Genetic inhibition of CARD9 accelerates the development of atherosclerosis in mice through CD36 dependent-defective autophagy 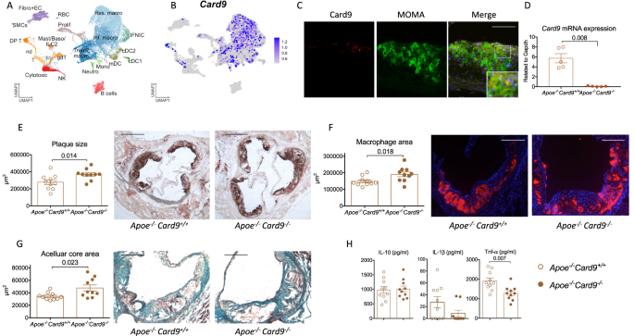Fig. 1:Global Card9deficiency accelerates atherosclerosis inApoe-/-mice. scRNA-seq analysis ofCard9transcript expression in murine arteries with 26,910 immune and non immune cells from the aorta of atherosclerotic mice (integrated analysis of 13 datasets).AUMAP representation of single-cell RNA-seq gene expression data and cellular lineage identification. (VSMCs vascular smooth muscle cells, Fibro+EC fibroblasts and endothelial cells, DP T double poisitive T cells, RBC red blood cells, Prolif proliferating cells, Mast/BAso/ILC2 mast cells, basophils and type 2 innate lymphoid cells, T T cells, NK natural killer cells, gdT gammadelta T cells, Neutro neutrophils, Mono monocytes, mDC mature dendritic cells, cDC1 and 2 classical dendritic cells 1 and 2, IFNIC type I interferon inducible cells, Trem2 macroTrem2hi/Foamy macrophages, Inf. Macro inflammatory macrophages, Res. Macro resident macrophages, nd not determined).BCard9 expression in single cells projected onto the UMAP plot.CCard9 (Red) and MOMA-2 (Green) immunofluorescent staining in plaques of 20-week oldApoe-/-mice (Representative of 7 atherosclerotic plaques). Scale bar 50 μm.DCard9mRNA expression by peritoneal macrophages isolated fromApoe-/-Card9+/+andApoe-/-Card9-/-mice (n= 5/group).Erepresentative photomicrographs and quantitative analysis of atherosclerotic lesions in the aortic sinus of maleApoe-/-Card9+/+andApoe-/-Card9-/-mice after 6 weeks of fat diet (2 experiments pooled,n= 10/group); Scale bar 200 μm.Frepresentative photomicrographs and quantitative analysis of macrophage accumulation (MOMA staining, red) in atherosclerotic lesions ofApoe-/-Card9+/+andApoe-/-Card9-/-mice after 6 weeks of fat diet (2 experiments pooled,n= 10/group); Scale bar 100 μm.GRepresentative photomicrographs and quantitative analysis of acellular area (Masson’s Trichrome) ofApoe-/-Card9+/+andApoe-/-Card9-/-mice after 6 weeks of fat diet (2 experiments pooled,n= 10/group); Scale bar 100 μm.HCytokine production (ELISA in the supernatant) by Lps/Ifnγ-stimulated splenocytes fromApoe-/-Card9+/+andApoe-/-Card9-/-mice (n= 10/group). Data are presented as mean values ±SD. Two-tailed Mann–Whitney test. Source data are provided as a Source Data file. Caspase recruitment-domain containing protein 9 (CARD9) is a key signaling pathway in macrophages but its role in atherosclerosis is still poorly understood. Global deletion of Card9 in Apoe -/- mice as well as hematopoietic deletion in Ldlr -/- mice increases atherosclerosis. The acceleration of atherosclerosis is also observed in Apoe -/- Rag2 -/- Card9 -/- mice, ruling out a role for the adaptive immune system in the vascular phenotype of Card9 deficient mice. Card9 deficiency alters macrophage phenotype through CD36 overexpression with increased IL-1β production, increased lipid uptake, higher cell death susceptibility and defective autophagy. Rapamycin or metformin, two autophagy inducers, abolish intracellular lipid overload, restore macrophage survival and autophagy flux in vitro and finally abolish the pro-atherogenic effects of Card9 deficiency in vivo. Transcriptomic analysis of human CARD9 -deficient monocytes confirms the pathogenic signature identified in murine models. In summary, CARD9 is a key protective pathway in atherosclerosis, modulating macrophage CD36-dependent inflammatory responses, lipid uptake and autophagy. Atherosclerosis is a chronic inflammatory disease of large and medium-sized arteries that develops in response to subendothelial retention and modification of ApoB containing low-density lipoproteins (LDL) [1] . Inflammatory activation of endothelial cells orchestrates the recruitment of different subsets of circulating leukocytes, notably monocytes, into the vascular wall. Recruited monocytes significantly contribute to the pool of intimal macrophages [2] , which promote the growth of atherosclerotic plaque after differentiation, activation and proliferation. Macrophage activation, an instrumental step in the development of atherosclerosis, is associated with the upregulation of pattern recognition receptors for innate immunity, including scavenger receptors (SR-A, CD36) and pathogen recognition receptors, such as Toll-like receptors (TLRs) and Dectin receptors [3] , [4] , [5] . A broad range of molecules and particles bearing danger-associated molecular patterns, including oxidized LDL (oxLDL), can be taken up by macrophages, leading ultimately to the formation of pro-inflammatory foam cells [6] . CD36 is an archetypal pattern recognition receptor that binds polyanionic ligands of both pathogen- and self-origin [7] including oxLDL [8] . CD36 forms a complex with the TLR TLR4-TLR6 heterodimer, which recognizes oxLDL and stimulates pro-inflammatory pathways, including the NLRP3 inflammasome activation responsible for proIL-1β. cleavage and IL-1β secretion [9] . A large body of evidence suggests that cumulative metabolic/inflammatory signals and impaired efferocytosis foster apoptosis and secondary necrosis of foam cells, which contributes to the growth of the necrotic core and progression of atherosclerosis [10] . However, the critical downstream pathways that drive both macrophage activation and conversion into foam cells are still poorly understood. Here, we investigated the role of Caspase recruitment-domain containing protein 9 (Card9), a key regulator of inflammation, in atherosclerosis. Card9 is an adapter protein that integrates pattern recognition receptor downstream signals in macrophages and dendritic cells [11] . Card9 is particularly involved in response to fungi via C-type lectin sensing, but also in response to bacteria by mediating nucleotide-binding oligomerization domain 2 (NOD2)-dependent p38/JNK signaling and TLR signaling [12] . Card9 is required to mount appropriate immune responses through the production of interleukin (IL)−6, IL-17A, IFN-γ, and IL-22, which can affect gut microbiota [13] , with potential impact on atherosclerosis [14] . The role of Card9 in inflammatory diseases is ambiguous, being pathogenic in post-ischemic cardiac remodeling [15] , but protective in experimental colitis [13] . In two recent studies, the role of CARD9 in atherosclerosis has been explored, but results reported contradictory findings. One study showed increased lesion size in chimeric Ldlr -/- Card9 -/- mice [16] , whereas the other found that deletion of haematopoietic Card9 did not affect atherosclerosis in chimeric Ldlr -/- mice under hyperglycaemic conditions [17] . Moreover, the underlying mechanisms linking Card9 engagement to atherosclerosis development remain largely unknown. Here, using several complementary approaches and state-of-the-art models, we show that Card9 signaling pathway in macrophages regulates cytokine production, lipid upload, and cell survival. Global, as well as hematopoietic deletion of Card9, markedly accelerates the development of atherosclerosis, independently of the adaptive immune system. Mechanisms of the pro-atherogenic effects of Card9 deficiency mainly involve CD36-dependent defective autophagy. Genetic invalidation of Card9 accelerates atherosclerosis in Apoe -/- mice To gain insight into the immune cells expressing Card9 , single-cell analysis of total cells from mouse atherosclerotic aortas (see methods) was performed (Fig. 1A, B and Supplementary Fig. 1 ). Card9 transcript was detected in myeloid cells, and macrophages in particular, including atherosclerosis-associated inflammatory and Trem2 hi /Foamy macrophages (Fig. 1A, B and Supplementary Fig. 1a, b ). Analysis of a second, independent scRNA-seq dataset of Ldlr -/- mouse atherosclerotic aortas [18] corroborated preferential detection of Card9 transcripts in myeloid cells, including macrophages (Supplementary Fig. 2 ). Immunofluorescence staining confirmed that Card9 was expressed in atherosclerotic lesions of Apoe -/- mice at both early (Supplementary Fig. 3a ) and advanced stages of atherosclerosis (Fig. 1C ), and mainly co-localized with MOMA + macrophages (Fig. 1C ). In vitro, Card9 expression in macrophages was induced by oxLDL (Supplementary Fig. 3b ). Fig. 1: Global Card9 deficiency accelerates atherosclerosis in Apoe -/- mice. scRNA-seq analysis of Card9 transcript expression in murine arteries with 26,910 immune and non immune cells from the aorta of atherosclerotic mice (integrated analysis of 13 datasets). A UMAP representation of single-cell RNA-seq gene expression data and cellular lineage identification. (VSMCs vascular smooth muscle cells, Fibro+EC fibroblasts and endothelial cells, DP T double poisitive T cells, RBC red blood cells, Prolif proliferating cells, Mast/BAso/ILC2 mast cells, basophils and type 2 innate lymphoid cells, T T cells, NK natural killer cells, gdT gammadelta T cells, Neutro neutrophils, Mono monocytes, mDC mature dendritic cells, cDC1 and 2 classical dendritic cells 1 and 2, IFNIC type I interferon inducible cells, Trem2 macro Trem2 hi /Foamy macrophages, Inf. Macro inflammatory macrophages, Res. Macro resident macrophages, nd not determined). B Card9 expression in single cells projected onto the UMAP plot. C Card9 (Red) and MOMA-2 (Green) immunofluorescent staining in plaques of 20-week old Apoe -/- mice (Representative of 7 atherosclerotic plaques). Scale bar 50 μm. D Card9 mRNA expression by peritoneal macrophages isolated from Apoe -/- Card9 +/+ and Apoe -/- Card9 -/- mice ( n = 5/group). E representative photomicrographs and quantitative analysis of atherosclerotic lesions in the aortic sinus of male Apoe -/- Card9 +/+ and Apoe -/- Card9 -/- mice after 6 weeks of fat diet (2 experiments pooled, n = 10/group); Scale bar 200 μm. F representative photomicrographs and quantitative analysis of macrophage accumulation (MOMA staining, red) in atherosclerotic lesions of Apoe -/- Card9 +/+ and Apoe -/- Card9 -/- mice after 6 weeks of fat diet (2 experiments pooled, n = 10/group); Scale bar 100 μm. G Representative photomicrographs and quantitative analysis of acellular area (Masson’s Trichrome) of Apoe -/- Card9 +/+ and Apoe -/- Card9 -/- mice after 6 weeks of fat diet (2 experiments pooled, n = 10/group); Scale bar 100 μm. H Cytokine production (ELISA in the supernatant) by Lps/Ifnγ-stimulated splenocytes from Apoe -/- Card9 +/+ and Apoe -/- Card9 -/- mice ( n = 10/group). Data are presented as mean values ±SD. Two-tailed Mann–Whitney test. Source data are provided as a Source Data file. Full size image To investigate the role of Card9 in this experimental setting, we generated Apoe -/- Card9 -/- mice. Card9 deficiency was confirmed by qPCR in peritoneal macrophages (Fig. 1D ) and by immunostaining of atherosclerotic plaques (Supplementary Fig. 4a ). Body weight was slightly increased in Card9- deficient mice, but no significant differences in plasma cholesterol levels were observed between male Apoe -/- Card9 +/+ and Apoe -/- Card9 -/- mice (Supplementary Fig. 4b, c ). At 8 weeks of age, animals were put on a high-fat diet for 6 weeks to accelerate plaque formation. Apoe -/- Card9 -/- mice showed a significant increase in atherosclerotic lesion size in the aortic sinus (368 ± 64 vs 278 ± 87. 10 3 μm 2 , P < 0.05; Fig. 1E ). Card9 deletion in Apoe -/- mice induced a switch toward a more inflammatory plaque phenotype with a significant increase in macrophage accumulation (Fig. 1F ) and necrotic core size (Fig. 1G ). Collagen content was increased in plaques of Apoe -/- Card9 -/- mice (Supplementary Fig. 4d ), but T cell accumulation was similar (Supplementary Fig. 4e ). Dampened systemic pro-inflammatory cytokine signature in Apoe -/- Card9 -/- mice Because Card9 is known to modulate cytokine production and T cell polarization [13] , we next investigated the immuno-inflammatory response in male Apoe -/- Card9 +/+ and Apoe -/- Card9 -/- mice. Leukocyte populations were analyzed by flow cytometry in both blood and spleen at sacrifice. We did not observe any significant difference in leukocyte percentages in blood between groups. We only found a slight increase in neutrophil and classical monocyte counts in the blood of Apoe -/- Card9 -/- mice, compared to control Apoe -/- Card9 +/+ mice (Supplementary Fig. 5 ). Splenocyte number was significantly higher in Card9 -deficient mice but the proportion of myeloid and lymphoid populations was not different between groups (Supplementary Fig. 6 ). Splenocytes from Apoe -/- Card9 -/- mice stimulated with IFN-γ and LPS produced less TNF-α (Fig. 1H ) than those from control mice, but the production of IL-10 and IL-1β was not different. We then purified splenic CD4 + T cells from control Apoe -/- Card9 +/+ and Apoe -/- Card9 -/- mice and performed functional tests. In vitro, the proliferation of CD4 + T cells from Apoe -/- Card9 -/- mice was significantly increased compared with control cells (Data non shown), and their production of IFN-γ and IL-17A was increased. There were no differences in IL-10 and IL-22 production (Supplementary Fig. 4f ). Hematopoietic Card9 deficiency increases atherosclerosis in Ldlr -/- mice To confirm our result in another mouse model of atherosclerosis and to specifically investigate the role of hematopoietic Card9, we performed bone marrow (BM) transplantation experiments using either Card9 +/+ or Card9 -/- BM cells to repopulate lethally irradiated female Ldlr -/- mice. We confirmed that Card9 gene expression was almost abolished in peritoneal macrophages of chimeric Ldlr -/- Card9 -/- (Fig. 2A ). Chimeric Ldlr -/- mice were then fed a high-fat diet for 8 weeks. We observed no difference in body weights (Fig. 2B ) or serum cholesterol levels (Fig. 2C ) between the 2 groups of chimeric mice. In blood, myeloid populations were not different between groups, but we observed a significant increase in circulating CD4 + T and B cell counts in chimeric Ldlr -/- Card9 -/- mice (Supplementary Fig. 7 ). As shown in Fig. 2 , hematopoietic Card9 deficiency was associated with a significant increase in lesion development compared with controls, in the thoracoabdominal aorta (Fig. 2D ), and in the aortic sinus (Fig. 2E ). In addition, Card9 deletion induced a more inflammatory plaque phenotype with a significant increase in both macrophage accumulation (Fig. 2F ) and necrotic core size (Fig. 2G ). We also observed an increase in collagen content in plaques of chimeric Ldlr -/- Card9 -/- mice (Supplementary Fig. 8a ). T cell accumulation in plaques was similar in the 2 groups (Supplementary Fig. 8b ). Stimulated splenocytes from Ldlr -/- Card9 -/- mice produced less TNF-α, IL-1β, and IL-10 than splenocytes from Ldlr -/- Card9 +/+ mice (Fig. 2H ). Splenic CD4 + T cells isolated from Ldlr -/- Card9 -/- mice produced less IL-17A than CD4 + T cells from control Ldlr -/- Card9 +/+ mice. IL-10, IFN-γ and IL-22 production was not affected in our experimental conditions (Supplementary Fig. 8c ). Fig. 2: Hematopoietic Card9 deficiency accelerates atherosclerosis in Ldlr -/- mice. A Card9 mRNA expression by peritoneal macrophages isolated from chimeric Ldlr -/- Card9 +/+ and Ldlr -/- Card9 -/- mice ( n = 5/group). B body weight at sacrifice after 8 weeks of fat diet ( n = 14/group). C plasma cholesterol levels at sacrifice after 8 weeks of fat diet ( n = 14/group). D representative photomicrographs and quantitative analysis of atherosclerotic lesions on the thoraco-abdominal aortas from chimeric female Ldlr -/- Card9 +/+ and Ldlr -/- Card9 -/- mice after 8 weeks of fat diet ( n = 7 Ldlr -/- Card9 +/+ and n = 6 Ldlr -/- Card9 -/- ); Scale bar 1 mm. E representative photomicrographs and quantitative analysis of atherosclerotic lesions in the aortic sinus of chimeric Ldlr -/- Card9 +/+ and Ldlr -/- Card9 -/- mice after 8 weeks of fat diet (2 experiments pooled, n = 14/group); Scale bar 200 μm. F representative photomicrographs and quantitative analysis of macrophage accumulation (MOMA staining, red) in atherosclerotic lesions of chimeric Ldlr -/- Card9 +/+ and Ldlr -/- Card9 -/- mice after 8 weeks of fat diet (2 experiments pooled, n = 14/group); Scale bar 100 μm. G Representative photomicrographs and quantitative analysis of acellular area (Masson’s Trichrome) of chimeric Ldlr -/- Card9 +/+ and Ldlr -/- Card9 -/- mice after 8 weeks of fat diet (2 experiments pooled, n = 14/group); Scale bar 100 μm. H Cytokine production (ELISA in the supernatant) by Lps/Ifnγ-stimulated splenocytes isolated from chimeric Ldlr -/- Card9 +/+ and Ldlr -/- Card9 -/- mice ( n = 5 Ldlr -/- Card9 +/+ and n = 6 Ldlr -/- Card9 -/- ); Data are presented as mean values ±SD. Two-tailed Mann–Whitney test. Source data are provided as a Source Data file. Full size image Gut microbiota unlikely contributed to the acceleration of atherosclerosis induced by Card9 deficiency Previous studies have shown that Card9 plays a critical role in gut microbiota homeostasis. Card9 -/- mice have been shown to display dysbiosis [19] , which has been implicated in atherosclerosis development [20] . To evaluate a potential impact of Card9-induced dysbiosis in our experimental conditions, we analyzed the bacterial microbiota was performed using 16S rRNA based sequencing. While there were no significant differences in alpha diversity between Apoe -/- Card9 +/+ and Apoe -/- Card9 -/- mice (Supplementary Fig. 9a, b ), beta diversity analysis showed a significant difference between the 2 groups, as demonstrated by the PCoA plot of Bray-Curtis distance (Supplementary Fig. 9c ). To determine which taxonomic groups accounted for these differences, we performed linear discriminant analysis with effect size (Lefse) [21] . Compared to Apoe -/- Card9 +/+ mice, Apoe -/- Card9 -/- mice displayed an increase in the pathobiont Helicobacter with a concomitant decrease in beneficial members of the Firmicutes phylum , including the order Clostridiales , as well as in Candidatus arthromitus , segmented filamentous bacteria. These bacteria are essential for Th17 maturation in the murine gut [22] , and in the genus Akkermansia , a genus associated with a lean body type and favorable metabolic outcomes [23] (Supplementary Fig. 9d ). Given the marked dysbiosis in Card9 -deficient Apoe -/- mice, we aimed to determine whether this dysbiosis was also observed in Ldlr -/- mice transplanted with Card9 -/- bone marrow cells. As found in Apoe -/- mice, 16S rRNA based sequencing showed no significant difference in alpha diversity among the 2 groups, but the beta diversity analysis showed significant differences in mice transplanted with Card9 -/- BM cells (Supplementary Fig. 9e, f ). Of note, because of transient aplasia and increased risk of sepsis chimeric Ldlr -/- mice received antibiotics during 14 days following lethal irradiation and BM cell transplantation. The administration of antibiotics caused marked changes in the microbiota in the 2 groups. In particular, at genus level, Parasutterella was increased in Ldlr -/- Card9 -/- mice and the sulfate-reducing bacteria Desulfovibrio was enhanced in Ldlr -/- Card9 +/+ mice. Only one bacterial family, Clostridiaceae_1 that was increased in Ldlr -/- Card9 +/+ mice, was concordantly altered in the two sets of experiments (Supplementary Fig. 9g–h ). Taken together, these data confirm an effect of the Card9 on the gut microbiota composition. However, the highly divergent microbiota composition between Apoe -/- and Ldlr -/ genetic backgrounds despite similar Card9 effects on atherosclerosis suggests that the gut microbiota was unlikely involved in the vascular phenotype induced by Card9 deficiency. Pro-atherogenic effect of Card9 deficiency is not dependent on adaptive immunity As described above, Card9 deficiency had major effects on CD4 + T cell proliferation and polarization. In order to evaluate the role of adaptive immunity in the acceleration of atherosclerosis observed in Card9 -deficient mice, we backcrossed Apoe -/- Rag2 -/- mice with Rag2 -/- Card9 -/- to generate athero-prone lymphocyte (T, B, NKT)-deficient Apoe -/- Rag2 -/- Card9 -/- mice. Eight-week old male control Apoe -/- Rag2 -/- Card9 +/+ and Apoe -/- Rag2 -/- Card9 -/- mice were fed a high-fat diet for 6 weeks. Card9 -deficiency was confirmed by qPCR in peritoneal macrophages (Fig. 3A ). There was no significant difference in body weight between groups (Fig. 3B ) but plasma cholesterol levels were slightly increased in Card9 -deficient mice (+17%, Fig. 3C ). Apoe -/- Rag2 -/- Card9 -/- mice exhibited a significant increase in atherosclerotic lesion size in the thoracoabdominal aorta (+69%, Fig. 3D ) and in the aortic sinus (+50%, Fig. 3E ). In addition, Card9 deletion in Apoe -/- Rag2 -/- mice induced a switch toward a more inflammatory plaque phenotype with increased macrophage accumulation (Fig. 3F ) and necrotic core size (Fig. 3G ). Stimulated splenocytes from Apoe -/- Rag2 -/- Card9 -/- mice produced less TNF-α, IL-1β, and IL-10 than those from Apoe -/- Rag2 -/- Card9 +/+ mice (Fig. 3H ). Altogether, these results suggest that the adaptive immune system was not involved in the pro-atherogenic effects of Card9 deficiency. Fig. 3: Card9 deficiency accelerates atherosclerosis in immunodeficient Apoe -/- Rag2 -/- mice. A Card9 mRNA expression by peritoneal macrophages isolated from male Apoe -/- Rag2 -/- Card9 +/+ and Apoe -/- Rag2 -/- Card9 -/- mice ( n = 6/group). B Weight at sacrifice after 6 weeks of fat diet (3 pooled experiments, n = 16–18/group). C plasma cholesterol levels at sacrifice after 6 weeks of fat diet (3 pooled experiments, n = 14 Apoe -/- Rag2 -/- Card9 +/+ and n = 16 Apoe -/- Rag2 -/- Card9 -/- ). D representative photomicrographs and quantitative analysis of atherosclerotic lesions on the thoraco-abdominal aorta of of Apoe -/- Rag2 -/- Card9 +/+ and Apoe -/- Rag2 -/- Card9 -/- mice after 6 weeks of fat diet ( n = 6 Apoe -/- Rag2 -/- Card9 +/+ and n = 7 Apoe -/- Rag2 -/- Card9 -/- ); E representative photomicrographs and quantitative analysis of atherosclerotic lesions in the aortic sinus of Apoe -/- Rag2 -/- Card9 +/+ and Apoe -/- Rag2 -/- Card9 -/- mice after 6 weeks of fat diet (3 experiments pooled, n = 14 Apoe -/- Rag2 -/- Card9 +/+ and n = 16 Apoe -/- Rag2 -/- Card9 -/- ); Scale bar 200 μm. F representative photomicrographs and quantitative analysis of macrophage accumulation (MOMA staining, red) in atherosclerotic lesions of Apoe -/- Rag2 -/- Card9 +/+ and Apoe -/- Rag2 -/- Card9 -/- mice after 6 weeks of fat diet (3 experiments pooled, n = 14 Apoe -/- Rag2 -/- Card9 +/+ and n = 16 Apoe -/- Rag2 -/- Card9 -/- ); Scale bar 100 μm. G Representative photomicrographs and quantitative analysis of acellular area (Masson’s Trichrome) of Apoe -/- Rag2 -/- Card9 +/+ and Apoe -/- Rag2 -/- Card9 -/- mice after 6 weeks of fat diet (3 experiments pooled, n = 14 Apoe -/- Rag2 -/- Card9 +/+ and n = 16 Apoe -/- Rag2 -/- Card9 -/- ); Scale bar 100 μm. H Cytokine production (ELISA) by Lps/Ifnγ-stimulated splenocytes isolated from Apoe -/- Rag2 -/- Card9 +/+ and Apoe -/- Rag2 -/- Card9 -/- mice ( n = 6/group). Data are presented as mean values ±SD. Two-tailed Mann–Whitney test. Source data are provided as a Source Data file. Full size image Card9 deficiency upregulates CD36 expression and increases foam cell formation Next, we speculated that the marked increase of acellular area in atherosclerotic plaques of Card9- deficient mice might be related to increased foam cell formation. To explore this hypothesis, we performed in vitro experiments investigating the uptake of oxidized LDL (ox-LDL) by BM-derived macrophages and their ability to accumulate intracellular lipids. 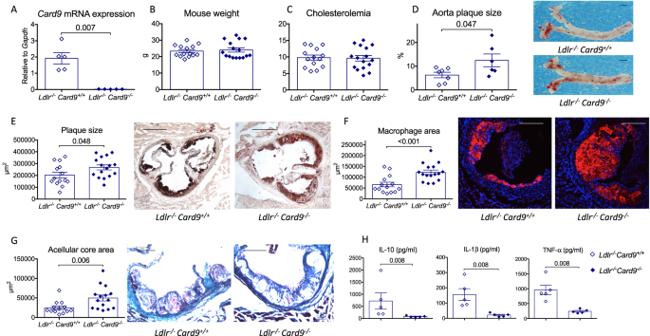Fig. 2: HematopoieticCard9deficiency accelerates atherosclerosis inLdlr-/-mice. ACard9mRNA expression by peritoneal macrophages isolated from chimericLdlr-/-Card9+/+andLdlr-/-Card9-/-mice (n= 5/group).Bbody weight at sacrifice after 8 weeks of fat diet (n= 14/group).Cplasma cholesterol levels at sacrifice after 8 weeks of fat diet (n= 14/group).Drepresentative photomicrographs and quantitative analysis of atherosclerotic lesions on the thoraco-abdominal aortas from chimeric femaleLdlr-/-Card9+/+andLdlr-/-Card9-/-mice after 8 weeks of fat diet (n= 7Ldlr-/-Card9+/+andn= 6Ldlr-/-Card9-/-); Scale bar 1 mm.Erepresentative photomicrographs and quantitative analysis of atherosclerotic lesions in the aortic sinus of chimericLdlr-/-Card9+/+andLdlr-/-Card9-/-mice after 8 weeks of fat diet (2 experiments pooled,n= 14/group); Scale bar 200 μm.Frepresentative photomicrographs and quantitative analysis of macrophage accumulation (MOMA staining, red) in atherosclerotic lesions of chimericLdlr-/-Card9+/+andLdlr-/-Card9-/-mice after 8 weeks of fat diet (2 experiments pooled,n= 14/group); Scale bar 100 μm.GRepresentative photomicrographs and quantitative analysis of acellular area (Masson’s Trichrome) of chimericLdlr-/-Card9+/+andLdlr-/-Card9-/-mice after 8 weeks of fat diet (2 experiments pooled,n= 14/group); Scale bar 100 μm.HCytokine production (ELISA in the supernatant) by Lps/Ifnγ-stimulated splenocytes isolated from chimericLdlr-/-Card9+/+andLdlr-/-Card9-/-mice (n= 5Ldlr-/-Card9+/+andn= 6Ldlr-/-Card9-/-); Data are presented as mean values ±SD. Two-tailed Mann–Whitney test. Source data are provided as a Source Data file. Interestingly, foam cell formation was significantly increased in Card9- deficient macrophages, compared with control macrophages, after 6 and 24 h of incubation with ox-LDL (Fig. 4A, B ). Total cholesterol and cholesterol ester content, after ox-LDL exposure, were significantly increased in macrophages from Apoe -/- Card9 -/- mice, confirming the intracellular cholesterol overload (Fig. 4C, D ). Next, we investigated the mechanisms that could drive lipid overload in the absence of Card9. We measured a significant increase in Abca1 , Abcg1 and Scarb1 mRNA levels in macrophages from Apoe -/- Card9 -/- mice exposed to ox-LDL, compared to those from Apoe -/- Card9 +/+ mice (Fig. 4E ). Cholesterol transfer to HDL and to ApoA1 was also enhanced in Apoe -/- Card9 -/- macrophages (Fig. 4F ). This finding highly suggests that increased foam cell formation in Card9 -deficient macrophages was not due to impaired cholesterol efflux. Next, we investigated the expression of scavenger receptors involved in lipid uptake. We found no difference in Msr1 mRNA content between groups but Cd36 mRNA levels were markedly increased in macrophages from Apoe -/- Card9 -/- mice exposed to ox-LDL (Fig. 4G ), which was confirmed at the protein level by immunofluorescent staining (Fig. 4H, I ). In agreement with our in vitro experiments, Cd36 mRNA levels were higher in aortas from Apoe -/- Card9 -/- mice, compared with control mice (Supplementary Fig. 10a ), as well as CD36+ macrophage numbers (Supplementary Fig. 10b ). Fig. 4: Card9 deficiency increased CD36 expression in macrophages and promotes lipid uptake and foam cell formation. A Representative photomicrographs and quantitative analysis ( B ) of Bodipy+ foam cells after incubation of BMDMs from Apoe -/- Card9 +/+ and Apoe -/- Card9 -/- mice with oxLDL during 6 and 24 h (2 pooled experiments, n = 8/group/timepoints), Scale bar 10 μm. C quantification of intracellular cholesterol content of BMDMs from Apoe -/- Card9 +/+ and Apoe -/- Card9 -/- mice after exposure to ox-LDL ( n = 6/group/timepoint). D Quantification of intracellular cholesterol ester of BMDMs from Apoe -/- Card9 +/+ and Apoe -/- Card9 -/- mice after exposure to ox-LDL at 3, 6, 12, and 24 h ( n = 6/group/timepoint). E Quantification of Abca1 and Abcg1 and Scarb1 mRNA expression in BMDMs from Apoe -/- Card9 +/+ and Apoe -/- Card9 -/- mice after stimulation with oxLDL ( n = 6/group). F Quantification of cholesterol efflux in presence of ApoAI or HDL ( n = 4/group). G Quantification of Mrs1 and Cd36 mRNAs in BMDMs from Apoe -/- Card9 +/+ and Apoe -/- Card9 -/- mice after stimulation with oxLDL ( n = 6/group). H , I representative immunostaining and quantification of Cd36 expression by BMDMs from Apoe -/- Card9 +/+ and Apoe -/- Card9 -/- mice after 24-h stimulation with ox-LDL ( n = 12 Apoe -/- Card9 +/+ and n = 22 Apoe -/- Card9 -/- ), Scale bar 10 μm. J cytokine production by BMDMs from Apoe -/- Card9 +/+ and Apoe -/- Card9 -/- mice after stimulation (ELISA in the supernatant, n = 5/group) and oxLDL exposure. K , L Flow cytometry quantification of AnnexinV+ BMDMs from Apoe -/- Card9 +/+ and Apoe -/- Card9 -/- mice after 24-h stimulation with oxLDL (100 μmol/l; n = 5/group). M , N representative photomicrographs and quantification of TUNEL+ cells in plaques from Apoe -/- Card9 +/+ and Apoe -/- Card9 -/- mice ( n = 10/group). Scale bar 20 μm. Data are presented as mean values ±SD. Two-tailed Mann–Whitney test. Source data are provided as a Source Data file. Full size image As intracellular lipid overload modulates cell phenotype, we investigated cytokine production by macrophages and apoptosis susceptibility. Interestingly, we observed that Card9 deficiency led to a phenotypic switch towards a more pro-inflammatory macrophage phenotype characterized by higher secretion of IL-1β and lower secretion of IL-10 following in vitro stimulation (Fig. 4J ). In addition, apoptosis was increased in macrophages from Apoe -/- Card9 -/- mice exposed to ox-LDL (Fig. 4K, L and Supplementary Fig. 10c ). On the same note we found that the number of TUNEL+ cells was increased in atherosclerotic plaques of Card9 -deficient mice (Fig. 4M, N and Supplementary Fig. 10d ), which might also account for the presence of large necrotic core in plaques of Apoe -/- Card9 -/- mice (Figs. 1 G, 2 G, and 3G ). Acceleration of atherosclerosis in Card9 deficiency is due to impaired autophagy The phenotype of Card9- deficient mice, in terms of size and composition of atherosclerotic plaques, as well as macrophage apoptosis susceptibility, resembled that of Atg5 fl/fl LysM Cre+/− Ldlr −/− mice that are characterized by impaired autophagy flux [24] . Interestingly, CD36, which was up-regulated in Card9- deficient mice, has been reported to participate in the regulation of autophagy in hepatocytes through AMPK downstream pathway [25] . Therefore, we next focused on the potential role of autophagy, a compensatory survival mechanism involved in atherosclerosis [26] , in the context of Card9 deficiency both in vitro and in vivo. Macrophages isolated from Apoe -/- Card9 +/+ and Apoe -/- Card9 -/- mice were cultured and stressed to activate autophagy. Interestingly, we found a significant decrease in AMPK phosphorylation in Card9- deficient macrophages (Fig. 5A ) but no difference in CHOP levels as well as Beclin-1 and LKB-1 phosphorylation (Supplementary Fig. 11 ). In addition, we found higher p62 protein content in macrophages from Apoe -/- Card9 -/- mice compared to Apoe -/- Card9 +/+ mice (Fig. 5A ). Confocal analysis of immunofluorescence staining of the p62 protein confirmed it was increased in the cytoplasm of unstimulated Card9 -deficient macrophages, and much more in the presence of oxLDL (Fig. 5B ). The p62 protein was co-localized with large inclusion bodies. LC3B dot size was significantly larger in the cytoplasm of Apoe -/- Card9 -/- macrophages, with specific aberrant colocalization with these large p62+ inclusion bodies (Fig. 5B ). P62+ inclusions bodies have been previously described in Atg5 -null macrophages [27] , which strongly supports impaired autophagy in the absence of Card9. The accumulation of p62 in Card9 -deficient macrophages was confirmed in vivo, as revealed by the higher number of p62+ MOMA+ macrophages in atherosclerotic plaques of Apoe -/- Card9 -/- mice in reference to plaques of Apoe -/- Card9 +/+ mice (Fig. 5C ). Next, we evaluated a pharmacological approach to restore autophagy treated with Metformin, a well-known activator of autophagy through AMPK stimulation [28] . In vitro, metformin treatment abolished the accumulation of p62+ protein in the Card9 -deficient macrophages and the formation of inclusion bodies (Fig. 5D ). In vivo, Apoe -/- Card9 +/+ and Apoe -/- Card9 -/- mice, under a high-fat diet, were treated or not with metformin during 6 weeks [28] . At sacrifice, there was no significant difference in body weight and in plasma cholesterol levels between Apoe -/- Card9 +/+ and Apoe -/- Card9 -/- groups treated with metformin (Supplementary Fig. 12a, b ). Metformin treatment abolished the acceleration of atherosclerosis observed in Card9 deficiency, with no difference in plaque size (Fig. 5E ), plaque composition (Fig. 5F, G ) and P62 accumulation (Fig. 5H ) between the 2 treated groups. Fig. 5: Pro-atherogenic effects of Card9 deficiency are mediated by impaired autophagy. A Quantitation of AMPK phosphorylation and p62 content in macrophages from from Apoe -/- Card9 +/+ ( n = 5) and Apoe -/- Card9 -/- mice ( n = 8) after exposure to oxLDL (western blot). B representative photomicrographs and quantitative analysis and of p62 (Red), LC3B (Green) content in macrophages from Apoe -/- Card9 +/+ and Apoe -/- Card9 -/- mice at baseline and after exposure to oxLDL ( n = 48 for p62 and n = 40 for LC3B). C Quantitative analysis and representative photomicrographs of p62 accumulation (Red) in MOMA-2+ macrophages (Green) in atherosclerotic lesions of Apoe -/- Card9 +/+ ( n = 10) and Apoe -/- Card9 -/- mice ( n = 12) after 6 weeks of fat diet (2 experiments pooled); Scale bar 200 μm. D representative photomicrographs and quantitative analysis and of p62 (Red), LC3B (Green) content in ox-LDL exposed macrophages from Apoe -/- Card9 +/+ and Apoe -/- Card9 -/- mice treated or not with metformin ( n = 48 for p62 and n = 40 for LC3B). E – H characterization of atherosclerotic lesions in the aortic sinus of male Apoe -/- Card9 +/+ ( n = 8 ) and Apoe -/- Card9 -/- mice ( n = 7) after 6 weeks of fat diet and treated by metformin. E representative photomicrographs and quantitative analysis of atherosclerotic lesions in the aortic sinus of Apoe -/- Card9 +/+ and Apoe -/- Card9 -/- mice after 6 weeks of fat diet and treated by metformin; Scale bar 200 μm. F representative photomicrographs and quantitative analysis of macrophage accumulation (MOMA staining, red) in atherosclerotic lesions of Apoe -/- Card9 +/+ and Apoe -/- Card9 -/- mice after 6 weeks of fat diet and treated by metformin; Scale bar 100 μm. G representative photomicrographs and quantitative analysis of acellular area (Masson’s Trichrome) of Apoe -/- Card9 +/+ and Apoe -/- Card9 -/- mice after 6 weeks of fat diet and treated by metformin; Scale bar 100 μm. H representative photomicrographs and quantitative analysis of p62 content (Green) in plaques of Apoe -/- Card9 +/+ and Apoe -/- Card9 -/- mice after 6 weeks of fat diet and treated by metformin; Scale bar 100 μm. Data are presented as mean values ±SD. Two-tailed Mann–Whitney test. Source data are provided as a Source Data file. Full size image Next, we used an addition complementary pharmacological approach to activate autophagy with rapamycin, an inhibitor of both mTORC1 and mTORC2 [29] . In vitro, rapamycin treatment restored autophagy flux, as shown by strong reduction of p62 protein accumulation in the cytoplasm of Card9 -deficient macrophages and an almost disparition of p62+ inclusion bodies (Fig. 6A, B ). In addition, rapamycin treatment abolished intracellular lipid overload (Fig. 6C ), and attenuated cell death susceptibility observed in Card9 -deficient macrophages (Fig. 6D ). To further validate the physiopathological relevance of our findings, Apoe -/- Card9 +/+ and Apoe -/- Card9 -/- mice were fed a high-fat diet for 6 weeks and received daily Rapamycin treatment. There was no difference in body weight and in plasma cholesterol levels between Apoe -/- Card9 +/+ and Apoe -/- Card9 -/- groups treated with rapamycin (Supplementary Fig. 12c, d ). Interestingly, rapamycin treatment abolished the pro-atherogenic effect of Card9 deficiency. Histological analysis revealed a significant decrease in atherosclerosis in the aortic sinus of rapamycin-treated Apoe -/- Card9 -/- mice , compared to rapamycin-treated Apoe -/- Card9 +/+ mice (Fig. 6D ). In addition, macrophage content and necrotic core size were also significantly reduced in atherosclerotic plaques of rapamycin-treated Apoe -/- Card9 -/- mice (Fig. 6F, G ), as well as the accumulation of p62 (Fig. 6H ). Fig. 6: Protective effects of rapamycin in vitro and in vivo. A , B representative photomicrographs and quantitative analysis of p62 (Red), LC3B (Green) content in oxLDL-exposed macrophages from male Apoe -/- Card9 +/+ and Apoe -/- Card9 -/- mice treated or not with rapamycin (200 mMol) ( n = 48 for p62 and n = 40 for LC3B). C quantification of intracellular cholesterol (total and ester) of BMDMs from Apoe -/- Card9 +/+ and Apoe -/- Card9 -/- mice after exposure to oxLDL with or without rapamycin (200 mMol) ( n = 5/group). D Flow cytometry quantification of necrosis (7AAD+ Annexin V+) susceptibility of macrophages from Apoe -/- Card9 +/+ and Apoe -/- Card9 -/- mice after 24-h stimulation with high concentration of oxLDL (100 μmol/l) without and with rapamycin (200 mMol; n = 5/group). E representative photomicrographs and quantitative analysis of atherosclerotic lesions in the aortic sinus of Apoe -/- Card9 +/+ and Apoe -/- Card9 -/- mice after 6 weeks of fat diet and treated by rapamycin ( n = 7/group); Scale bar 200 μm. F representative photomicrographs and quantitative analysis of macrophage accumulation (MOMA staining, red) in atherosclerotic lesions of Apoe -/- Card9 +/+ and Apoe -/- Card9 -/- mice after 6 weeks of fat diet and treated by rapamycin ( n = 7/group; Scale bar 100 μm). G representative photomicrographs and quantitative analysis of acellular area (Masson’s Trichrome) of Apoe -/- Card9 +/+ and Apoe -/- Card9 -/- mice after 6 weeks of fat diet and treated by rapamycin ( n = 7/group; Scale bar 100 μm). H representative photomicrographs and quantitative analysis of p62 content (green) in plaques of Apoe -/- Card9 +/+ and Apoe -/- Card9 -/- mice after 6 weeks of fat diet and treated by rapamycin ( n = 7/group; Scale bar 100 μm.). Data are presented as mean values ±SD. Two-tailed Mann–Whitney test. Source data are provided as a Source Data file. Full size image Card9 deficiency-mediated acceleration of atherosclerosis is dependent on CD36 To address the direct role of CD36, we generated Cd36 -deficient Card9 +/+ and Card9 -/- mice. Following in vitro challenge, AMPK phosphorylation (Fig. 7A ), p62 accumulation (Fig. 7B ), lipid uptake (Fig. 7C and supplementary Fig. 13a, b ) and cell death susceptibility (Fig. 7D ) were not different between macrophages from Cd36 -/- Card9 +/+ and Cd36 -/- Card9 -/- mice. Furthermore, increased production of IL-1β observed in Card9 -/- macrophages was also abolished in the absence of Cd36 (Fig. 7E ). Fig. 7: Pro-atherogenic effect of hematopoietic Card9 deficiency was abolished in the absence of Cd36. A representative blots and quantification of AMPK phosphorylation on BM-derived macrophages from Cd36 -/- Card9 +/+ and Cd36 -/- Card9 -/- macrophages after exposure to oxLDL ( n = 6/group/condition). B Quantitative analysis and representative photomicrographs of P62 accumulation in macrophages from Cd36 -/- Card9 +/+ and Cd36 -/- Card9 -/- macrophages after 8-h exposure to oxLDL, Scale bar 100 μm ( n = 6/group/condition). C quantification of intracellular Cholesterol of BM-derived macrophages from Cd36 -/- Card9 +/+ and Cd36 -/- Card9 -/- mice after 3 and 6 h exposure to ox-LDL ( n = 5/group/timepoint). D Flow cytometry quantification of Annexin V+ apoptotic BM-derived macrophages from Cd36 -/- Card9 +/+ and Cd36 -/- Card9 -/- mice after 24-h stimulation with high concentration of oxLDL (50 μmol/l; Baseline n = 6/group, OxLDL n = 7 Cd36 -/- Card9 +/+ and n = 8 Cd36 -/- Card9 -/- ). E Cytokine production by BMDMs from Cd36 -/- Card9 +/+ and Cd36 -/- Card9 -/- mice after stimulation (ELISA in the supernatant, n = 6/group). F Cd36 mRNA expression in the spleen from Ldlr -/- mice and chimeric Ldlr -/- Cd36 -/- Card9 +/+ and Ldlr -/- Cd36 -/- Card9 -/- mice ( n = 20/10/10). G Card9 mRNA expression in the spleen from Ldlr -/- mice and chimeric Ldlr -/- Cd36 -/- Card9 +/+ and Ldlr -/- Cd36 -/- Card9 -/- mice ( n = 20/10/10). H – K characterization of chimeric male Ldlr -/- Cd36 -/- Card9 +/+ ( n = 10) and Ldlr -/- Cd36 -/- Card9 -/- mice ( n = 11). H cholesterolemia in chimeric mice at sacrifice. I representative photomicrographs and quantitative analysis of atherosclerotic lesions in the aortic sinus of chimeric Ldlr -/- Cd36 -/- Card9 +/+ and Ldlr -/- Cd36 -/- Card9 -/- mice after 8 weeks of fat diet; Scale bar 200 μm. J representative photomicrographs and quantitative analysis of macrophage accumulation (MOMA staining, red) in atherosclerotic lesions of chimeric Ldlr -/- Cd36 -/- Card9 +/+ and Ldlr -/- Cd36 -/- Card9 -/- mice after 8 weeks of fat diet; Scale bar 100 μm. K Representative photomicrographs and quantitative analysis of acellular area (Masson’s Trichrome) of chimeric Ldlr -/- Cd36 -/- Card9 +/+ and Ldlr -/- Cd36 -/- Card9 -/- mice after 8 weeks of fat diet; Scale bar 100 μm. Data are presented as mean values ±SD. Two-tailed Mann–Whitney test. Source data are provided as a Source Data file. Full size image To investigate the effect of Card9 deficiency on atherosclerosis in the absence of CD36, we performed BM transplantation experiments using either Cd36 -/- Card9 +/+ or Cd36 -/- Card9 -/- littermate BM to repopulate lethally irradiated male Ldlr -/- mice. After 4 weeks of recovery and additional 8 weeks of high-fat diet, animals were sacrified. We confirmed that Cd36 and Card9 gene expression was almost abolished in the spleen (Fig. 7F, G ) and in peritoneal macrophages of chimeric Ldlr -/- (Supplementary Fig. 13c ). Cholesterol levels were not different between both groups (Fig. 7H ). Atherosclerosis plaque size and composition were no longer different between Ldlr -/- Cd36 -/- Card9 +/+ and Ldlr -/- Cd36 -/- Card9 -/- chimeric groups (Fig. 7I, K ), indicating that increased expression of CD36 was directly responsible for increased atherosclerosis in Card9 -deficient animals. CARD9-related pathways in human In order to evaluate the clinical relevance of our experimental results, we compared the transcriptomic profile of blood monocytes from CARD9 -deficient patients ( n = 3, 2 males and 1 female) with those of controls ( n = 4, 2 males and 2 females) (Fig. 8A and Supplementary data 1a, b ). Genetic investigations in CARD9 -deficient patients identified a homozygous c.865C > T in exon 6 of CARD9 leading to a premature stop codon at position 289 (p.Q289*) ( n = 2, 1 male and 1 female) and a homozygous c.52 C > T missense mutation in exon 2 of CARD9, resulting in the replacement of the arginine in position 18 with a tryptophan residue (p.R18W) ( n = 1 female) [30] , [31] , [32] . Differential analysis of these RNA-Seq revealed 256 differentially expressed genes (Fig. 8B ): 211 were up-regulated and 45 were down-regulated in CARD9 -deficient patients. Up-regulated genes included inflammatory cytokines, such as IL-1β [log2(FC) = 2.2, adjusted p -value = 0.035] and IL-6 [log2(FC) = 4.3, adjusted p -value = 1.52e-05] (Fig. 8C ). In gene set enrichment analysis (GSEA), several pathways previously identified in murine models had significant enriched score: apoptosis (34 pathways, 330 genes), autophagy (1 pathway, 1 gene), atherosclerosis (2 pathways, 69 genes), NF-κB signaling (1 pathway, 25 genes) and TNFα signaling pathway (1 pathway, 20 genes) (Fig. 8D and detailed selected pathways and core enrichment genes in Supplementary data 2 ). Fig. 8: CARD9 related pathways in human. A protocol to obtain transcripts after isolation of monocytes from controls and CARD9 -deficient patients. B Volcano-plot of the differentially expressed genes between monocytes from patients with CARD9 mutation and control patients. Red dots represent up-regulated genes and blue dots down-regulated genes (adjusted p -value < 0.05). C Heatmap of mean expression in each patient of the leading edge genes contributing to the enrichment of indicated pathways in the GSEA. Immunofluorescent micrograph of human healthy ( D ) and atherosclerotic ( E ) carotid artery sections stained for CARD9 (green), α-actin + smooth muscle (red) or CD68 (red) showing that CARD9 was strongly expressed by cells that engulf lipids and cholesterol crystals and of giant lipid-laden foam cells but not by smooth muscle cells. Magnitude X20 (D), X2.5 (E), X40 (E) (2 Pooled experiments, n = 6/staining). F CARD9 expression in 10,934 total human atherosclerotic coronary artery cells from 4 patients (data from Wirka et al. [33] ) with UMAP representation of single-cell RNA-seq gene expression data (left) and cellular lineage identification (right) where CARD9 expression in single cells projected onto the UMAP plot. (For clarity, expression cutoff have been applied and cells with detectable Card9/CARD9 transcripts were brought to the front of the plot). Full size image Finally, we examined CARD9 expression in atherosclerotic plaques from human carotid arteries. CARD9 was not detected in normal aorta (Supplementary Fig. 14a ). However, CARD9 was detected in fatty streak lesions (Fig. 8D ) and in lipid-rich areas surrounding the necrotic core of advanced atherosclerotic plaques (Fig. 8E ). CARD9 expression was higher in atheromatous plaques than in fibrous lesions (Supplementary Fig. 14b ). Fluorescent staining confirmed that CARD9 expression was mostly confined to CD68 + intimal macrophages (Fig. 8D, E ), and analysis of previously published single-cell RNA-seq [33] revealed CARD9 mRNA expression specifically in macrophages from atherosclerotic human coronary arteries (Fig. 8F and Supplementary Fig. 15a–d ). In an integrated single-cell analysis of human mononuclear phagocytes in atherosclerosis [34] , CARD9 was detected in all the major plaque macrophage subsets (Supplementary Fig. 15e–g ). Using several in vitro and in vivo complementary approaches, we demonstated that Card9 deficiency significantly accelerated atherosclerosis in mice throughout the aorta (aortic sinus, ascending and descending aorta) and induced a more inflammatory plaque phenotype, characterized by increased macrophage infiltration and necrotic core size. Card9 -deficient macrophages are characterized by increased pro-inflammatory cytokine release, enhanced lipid uptake and elevated cell death susceptibility (Supplementary Fig. 16 ). Such pro-atherogenic phenotype resulted from CD36-mediated impaired autophagy, since this was reversed by Cd36 gene deletion and by autophagy-inducing treatments with rapamycin and metformin. Importantly, the human relevance of our findings in mice was confirmed using transcriptomic analysis of monocytes isolated from extremely rare CARD9 -deficient patients and ScRNA seq analysis in human atherosclerotic plaques. The role of CARD9 in atherosclerosis still remains debated. In two recent studies, one reported increased lesion size in chimeric Ldlr -/- Card9 -/- mice [16] , whereas the other found that deletion of haematopoietic Card9 did not affect the atherosclerosis in chimeric Ldlr -/- mice under hyperglycaemic conditions [17] . In our study, we provided strong evidence that Card9 deficiency promoted atherosclerosis. We confirmed this finding in two different atheroprone models, Apoe -/- mice and chimeric Ldlr -/- mice under high-fat diet. The pro-atherogenic role of Card9 deficiency was not dependent on gender as we observed similar accelerated vascular disease in both male Apoe -/- and female chimeric Ldlr -/- mice with Card9 deficiency. The acceleration of atherosclerosis, which is known to be an inflammatory disease, in the absence of Card9 might be counterintuitive since Card9 is a downstream adapter of fungal- and bacteria-induced activation of TLRs, as well as activation of ITAM-containing non-TLRs and Dectin-1 [35] , [36] . Card9 engagement and Card9-Bcl-10-MALT1 complex formation lead to NF-κB transcription and subsequent secretion of pro-inflammatory cytokines [37] . Decreased spleen production of TNF-α is consistent in all murine models and in line with previous studies [35] . The effect of Card9 deficiency on IL-1β production is more complex. We found decreased IL-1β production by stimulated mixed immune cells in the spleen, but higher production by murine Card9 -/- macrophages as well as higher IL-1β transcripts in monocytes from CARD9 -deficient patients. In the context of Salmonella infection, it has also been reported that CARD9 negatively regulates IL-1β by fine-tuning pro-IL-1β expression, SYK-mediated NLRP3 activation and repressing inflammasome-associated caspase-8 activity [38] . Higher production of IL-1β might be involved, at least in part, in the acceleration of atherosclerosis in Apoe -/- Card9 -/- mice and might be due to increased CD36 expression. Liu et al. have shown that CD36 promoted the expression of NLRP3 and consecutive IL-1β production through ROS generation in ox-LDL-stimulated macrophages [39] . In our study, we found that Card9 deficiency had significant effects on the adaptive immune system and particularly on T cell polarization. We observed discrepancies in cytokine production by CD4 + T cells between male Apoe -/- and female chimeric Ldlr -/- , which could be due to gender or background difference, Apoe having by itself immune-modulatory functions [40] . In chimeric Ldlr -/- mice, Card9 -deficient CD4 + T cells produced less IL-17A than control CD4 + T cells, which is consistent with previous studies in normocholesterolemic mice [13] . However, our findings of increased atherosclerosis in immune-deficient Apoe -/- Rag2 -/- Card9 -/- mice ruled out the possibility that the acceleration of atherosclerosis in the absence of Card9 was mediated by a modulation of the adaptive immune system. Given the marked increase in aortic atherosclerosis in the absence of hematopoietic Card9 and the colocalization between Card9+ macrophages and lipid-rich areas in both mouse and human plaques, we then focused on the role of Card9 in macrophage foam cell formation. We found a marked increase in ox-LDL uptake and lipid accumulation in Card9 -/- macrophages. Among the receptors that govern foam cell formation in macrophages, Card9 deletion selectively increased both Cd36 gene expression and cell surface protein levels, in vitro, as well as in vivo in plaque macrophages. The effect of Card9 deficiency on the upregulation of CD36 expression and lipid uptake might account for the accelerated atherosclerosis in Card9 -deficient mice. Several studies have previously reported a pro-atherogenic role of CD36 in Apoe -/- [41] and Ldlr -/- mice [42] . We reported increased apoptosis susceptibility of Card9 -/- macrophages exposed to ox-LDL, which is consistent with the increase number of TUNEL+ cells found in plaques of Apoe -/- Card9 -/- mice. Apoptosis susceptibility of Ca rd9 -deficient macrophages might be due to intracellular lipid overload. In the context of atherosclerosis, other mechanisms, including autophagy, could account for enhanced apoptosis susceptibility of macrophages in the absence of Card9. Notably, we found that autophagy was impaired in cultured Card9 -deficient macrophages, as well as in atherosclerotic plaques of Apoe -/- Card9 -/- mice, as shown by the accumulation of p62 accumulation. Confocal analysis revealed that the p62 protein accumulated in large inclusion bodies with LC3B. These inclusion bodies that are p62-enriched polyubiquitinated protein aggregates, have been previously described in the context of impaired autophagy [27] . These observations highly suggested that Card9 deficiency impaired autophagy flux, but the exact molecular mechanisms requires further investigation. Ohman et al. previously suggested a link between the Card9 signaling pathway and autophagy, and found that Curdlan, an activator of the Dectin-1 receptor, induced LC3I conversion into LC3II in cultured macrophage [43] . More recently, Rubicon, a Beclin-1-binding partner, was identified as a physiological feedback inhibitor of Card9-BCL10-MALT1-mediated PRR signaling [44] . Impaired autophagy has also been shown to promote atherosclerosis. Autophagy blockade in LysMCre + Atg5l ox/lox Ldlr -/- mice led to increased lesion size and larger necrotic core [24] , which phenocopies the genetic loss of Card9 in Apoe -/- mice. Our study showed that impaired autophagy in Card9 -deficient macrophages was mediated, at least in part, by AMPK blockade. We focused on AMPK because CD36 is known to inhibit AMPK phosphorylation [25] , [45] and also because AMPK is an upstream regulator of autophagy through several mechanisms, including Ulk1 activation [46] and mTORC1 inhibition [47] . In Card9 -deficient macrophages, oxLDL-induced AMPK phosphorylation was abolished and P62 protein accumulated in cell cytoplasm. Interestingly, AMPK phosphorylation and autophagy were restored in Cd36 -/- Card9 -/- cells, supporting a critical role of CD36 in the regulation of autophagy and subsequently atherosclerotic plaque development. Rapamycin and metformin, two pharmacological activator of autophagy, respectively through mTOR blockade and AMPK activation [29] , restored in vitro autophagy flux in Card9 -deficient macrophages, with a strong reduction of p62+ inclusion bodies formation. In vivo, both treatment abolished the pro-atherogenic effect of Card9 deficiency and reduced p62 accumulation in atherosclerotic lesions. As rapamycin and metformin have several molecular targets, it cannot be ruled out that some of their anti-atherogenic effects were independent of their effect on autophagy. Experiments performed in Cd36 -/- animals confirmed that CD36 upregulation was involved in the acceleration of atherosclerosis in Card9 -/- animals. However, how the two functions of CD36 (lipid uptake versus autophagy) contribute to the pro-atherogenic impact of Card9 deficiency remains unknown. Addressing this issue is very challenging because autophagy, by itself, can regulate Cd36 levels [48] . Finally, in our study, cholesterol efflux was not impaired in Card9 -deficient macrophages suggesting that autophagy-independent mechanisms such as neutral lipolysis [49] , [50] were activated in Card9 -/- macrophages to limit lipid overload. Finally, given the marked differences in the profiles of gut microbiota between Apoe -/- and Ldlr -/- models, but the very similar pro-atherogenic effects of Card9 deficiency in these two murine models of atherosclerosis, it is unlikely that these vascular effects were due to Card9-associated dysbiosis. However, in the absence of microbiota transfer experiments, a contribution of gut dysbiosis in the vascular phenotype cannot be definitively ruled out. Altogether, our studies identify CARD9 as a major protective pathway in the development and complications of atherosclerosis. Pro-apoptotic and pro-atherogenic effects of Card9 deficiency are mediated by CD36-dependent defective autophagy that can be reversed by rapamycin and metformin. Animals Experiments were conducted according to the guidelines formulated by the European Community for experimental animal use (L358-86/609EEC) and were approved by the Ethical Committee of INSERM and the French Ministry of Agriculture (agreement A75-15-32). Mouse breeding occurred in our animal facility in accordance with local recommendations. Animals were provided with food and water ad libitum . All the animals were maintained under identical standard conditions (housing, regular care and high-fat diet). Mice were maintained in isolated ventilated cages under specific pathogenfree conditions. Before euthanasia by cervical dislocation, animals were anesthetized with isoflurane (3% in oxygen). Card9 -/- and Rag2 -/- Card9 -/- mice (null for the Card9 gene), have been generated by Dr. Harry Sokol (Centre de Recherche Saint-Antoine UMR_S 938, Paris, France) [13] . They were backcrossed for over 10 generations into a C57BL/6 J background. Apoe -/- Card9 -/- and Apoe -/- Rag2 -/- Card9 -/- mice have been generated in our lab and males were used for atherosclerosis studies. Cd36 -/- mice (null for the Cd36 gene) C57bl/6 Cd36 -/- mice were generated in Dr. Roy Silverstein’s laboratory (Febbraio et al. JBC 1999) and were crossed with Card9 -/- mice to generate Card9 -/- Card36 -/ - mice. Ten-week old female C57BL/6 J Ldlr -/- mice were subjected to medullar aplasia by lethal whole-body irradiation (9.5 grays). The mice were repopulated with an intravenous injection of bone marrow (BM) cells isolated from femurs and tibias of sex-matched C57BL/6 J Card9 -/- mice or Card9 +/+ littermates. After 4 weeks of recovery, mice were fed a pro-atherogenic high-fat diet containing 15% fat, 1.25% cholesterol, and 0% cholate for 8 weeks. During the first 14 days following BM cell transfer, animals were administered an antibiotic in their drinking water (Baytril®, Enrofloxacine). Ten-week old male C57BL/6J Ldlr -/- mice were subjected to medullar aplasia by lethal whole-body irradiation (9.5 grays). The mice were repopulated with an intravenous injection of bone marrow (BM) cells isolated from femurs and tibias of sex-matched C57BL/6 J Cd36 - /- Card9 +/+ mice or Cd36 - /- Card9 -/- littermates. After 4 weeks of recovery, mice were fed a pro-atherogenic high-fat diet containing 15% fat, 1.25% cholesterol, and 0% cholate for 8 weeks. Human carotid plaques Formalin-fixed and paraffin-embedded arterial tissue sections were used after antigen retrieval by heating in microwave oven in Tris/EDTA buffer pH9 (Dako). buffer. For single labeling, CARD9 rabbit polyclonal antibody (Abcam, Cambridge, UK) was used at 1:500 dilution, incubated for 1 h and revealed using ABC-peroxidase technique (Vector Laboratories, Burlingame, CA, USA). For double labeling, the sections were first incubated with mouse monoclonal anti-CD68 antibodies diluted at 1:50 (to detect macrophages) or anti-α smooth muscle actin antibodies diluted at 1:100 (to detect smooth muscle cells), both from Dako-Agilent (Trappes, France). Sections were then incubated with species-specific secondary antibodies (1:500 dilution, 45 min at room temperature) conjugated to AlexaFluor 488 or 594 (Fischer Scientific) and mounted on microscope slides using the Prolong Antifade Diamond kit (Thermofisher). Image acquisition was performed on a laser scanning confocal microscope (Leica TCS SP8, Leica Microsystems). Human ethics Our research complies with all relevant ethical regulations for all the human samples used. Immunostaining studies were performed on arteries obtained after surgery (Ethical Committee CPP Ile de France 2013-13-19) and written informed consent was obtained. Protein of plaques were from the Athero-Express study, a longitudinal vascular biobank study in which participants provided written informed consent, and the study was approved by the Medical Ethics Committee of the University Medical Center Utrecht (NL45885.041.13, METC 13/597, Medical Ethical Committee of University). Blood monocytes were obtained from a longitudinal biobank study in which participants provided written informed consent, and the study was approved by the ethical Committee for the Protection of Human Subjects in Biomedical Research (Inserm N° C10-14). Pharmacological in vivo treatment Eight-week old male Apoe -/- Card9 +/+ and Apoe -/- Card9 -/- mice were treated with daily intraperitoneal injections of rapamycin (4 mg/kg body weight) for 6 weeks and were put on a high-fat diet. Eight-week old male Apoe -/- Card9 +/+ and Apoe -/- Card9 -/- mice were treated with metformin (300 mg/kg body weight, drinking water) for 6 weeks and were put on a high-fat diet. Extent and composition of atherosclerotic lesions Plasma cholesterol was measured using a commercial cholesterol kit (DiaSys® Cholestérol FS*). Quantification of lesion size was standardized [51] . Briefly, the basal half of the ventricles and the ascending aorta were perfusion-fixed in situ with 4% paraformaldehyde, then transferred to a PBS-30% sucrose solution, embedded in frozen OCT and stored at −80 °C. Serial 10-μm sections of the aortic sinus with valves (80 per mouse) were cut on a cryostat [52] . One section out of 5 was used for plaque size quantification after Oil red O staining. In total, 16 sections spanning over 800 μm of the aortic root were used to determine the mean lesion area for each mouse. After PBS flushing, the aorta from the root to the iliac bifurcation was removed and fixed with 10% neutral-buffered formalin. After thorough PBS washing, the adventitial tissue was removed and the aorta was longitudinally opened to expose the luminal surface for en-face visualization of atherosclerotic lesions after Oil Red O staining. Quantification of Oil Red O positive surface area was performed by a blinded operator. Aortic collagen content was detected using Sirius red staining. Necrotic core surface was quantified after Masson’s Trichrome staining. At least 4 sections per mouse were examined for each immunostaining, and appropriate negative controls were used. Morphometric studies were performed using Histolab software (Microvisions) [53] . For immunostaining on mouse atherosclerotic plaques, we used antibodies raised against Card9 (AA 274-530), MOMA-2 (macrophage detection, MAB1852, Merck Milllipore®) and CD3 (T cell detection, A0452, Dako®) [53] . TUNEL (Terminal dUTP nick end-labeling) staining was performed using In Situ Cell Death Detection Kit (histochemistry staining) and TMR Red kit (Fluorescent staining) (Roche). The investigators were blinded to group allocation during data collection and analysis. Splenocyte culture Splenocytes were cultured in RPMI 1640 supplemented with Glutamax, 10% fetal calf serum (FCS), 0.02 mM β-mercaptoethanol and antibiotics. For cytokine measurements, splenocytes were stimulated with LPS (1 μg/ml) and IFN-γ (100 UI/ml) for 24 h. IL-1β, IL-10 and TNF-α production in the supernatants were measured using specific ELISA immunoassay kits (BD Biosciences). Spleen cell recovery and purification Spleen cells were purified according to standard protocols as follows. CD4 + T cells were negatively selected using a cocktail of anti-CD8a, anti-CD11b, anti-CD45R, anti-DX5, anti-ter 119 antibody-coated magnetic beads, yielding CD4 + cells with >95% purity (Miltenyi Biotech). CD11c + cells were positively selected with biotin-conjugated anti-CD11c mAb (7D4, PharMingen) and captured with streptavidin microbeads (Miltenyi Biotec) followed by 2 consecutive magnetic cell separations using LS columns (Miltenyi Biotec), yielding CD11c + cells with >80% purity. CD4 + T cell culture and cytokine assays Cells were cultured in RPMI 1640 supplemented with Glutamax, 10% FCS, 0.02 mM β-mercaptoethanol and antibiotics. For cytokine measurements, CD4 + T cells were cultured at 1 × 10 5 cells/well for 48 h in anti-CD3-coated microplates (5 μg/ml). In some experiments, CD4 + T cells were stimulated with purified soluble CD3-specific antibody (1 μg/ml, Pharmingen) in the presence of antigen-presenting cells that were purified on CD11c-coated magnetic beads (Miltenyi Biotech). Secretion of IL-17A, IL-22, IL-10, and IFN-γ secretion in the supernatants was measured using analyte-specific ELISAs (BD Biosciences and R&D Systems). T cell proliferation was measured using the Quick Cell proliferation Assay Kit II (Abcam). Macrophage experiments Primary macrophages were derived from mouse BM cells (BMDMs). Tibias and femurs of C57Bl6/J male mice were dissected and their marrow flushed out. Cells were grown in RPMI 1640 medium, 10% FCS, and 15% Macrophage–Colony-Stimulating Factor (M-CSF)-rich L929-conditioned medium for 7 days at 37 °C. To analyze oxidized LDL uptake, BMDMs were exposed to human oxidized LDL (25μg/ml) for 24 h (see oxidation method below). Cells were then washed, fixed and stained using Bodipy (493/503, Thermofischer Scientific D3922). Foam cells were quantified blindly on 6–8 fields and the mean was recorded. To analyze apoptosis susceptibility, macrophages were incubated with OxLDL (200 μg/ml) for 6, 12, and 24 h. Apoptosis was determined by independent experiments using Annexin V- (FITC) apoptosis detection kit with 7-AAD (PerCP) (BD Biosciences) according to the manufacturer’s instructions. Intracellular cholesterol (total and ester) quantification was done using Amplex® Red Cholesterol Assay Kit (Invitrogen A12216). For cytokine measurements, BM-derived macrophages were exposed to human oxLDL (25 μg/ml) and stimulated with LPS (1 μg/ml) for 24 h. Cytokine production in the supernatants were measured using specific ELISA immunoassay kits (BD Biosciences). Immunofluorescence on macrophages BM-Derived macrophages were fixed in ice-cold methanol, then washed twice in PBS. Cells were permeabilized with TBS + 0,1% triton for 10 min, then non-specific epitopes were blocked in TBS + 0,1% tween + 3% BSA for 20 min. Primary antibodies diluted in blocking buffer were incubated overnight at 4 °C. The following antibodies were used: Guinea-pig anti-P62 (Progen, GP62-C) and Rabbit anti-LC3B (Cell signaling technology, #43566). After washes in TBS + 0,1% tween, cells were incubated with alexa-568 donkey anti-guinea-pig and alexa-488 donkey anti-rabbit secondary antibodies (Invitrogen) for 2 h at room temperature. After incubation, cells were washed, nuclei were stained with Hoechst and slides were mounted with ibidi fluorescent mounting medium. Images were acquired on a Leica SP8 confocal with lightning super resolution module. Quantifications were done with ImageJ (NIH) using semi-automatic macros. Briefly, cells were manually circled to create ROI, then for each staining a threshold was applied and quantification of the number of particles, mean area of particles and area of ROI was measured using “Analyze particle”. For P62, inclusion bodies were defined as particles with area >100px. Macros are available upon request. Experiments were done in 4 replicates. For LC3+ dots per cell, 25 to 47 cells per condition were quantified and for P62+ inclusion bodies, 20 to 53 cells per condition were quantified. Cholesterol efflux assays BMDMs were obtained by differentiation of BM cells in Dulbecco’s modified Eagle medium (DMEM) supplemented with 10% fetal bovine serum, 2 mM glutamine, 20% L929 cell-conditioned media (as a source of M-CSF), and penicillin-streptomycin for 5 days. BMDMs were loaded with 50 µg/ml [3H]cholesterol-labeled acetylated LDL (acLDL, 1 µCi/mL) for 48 h in serum-free DMEM supplemented with 50 mM glucose, 2 mM glutamine, 0.2% BSA (RGGB), and 100 µg/ml penicillin / streptomycin. The labeling medium was then removed and cells were washed twice in PBS and then equilibrated in RGGB for additional 16–24 h. To measure cholesterol efflux, cells were incubated 4 h at 37 °C in the presence of 60 µg/ml lipid-free apoAI (Sigma), or 30 µg/ml HDL-PL (density = 1.063–1.21 g/ml), isolated from normolipidemic plasma by preparative ultracentrifugation, as cellular cholesterol acceptor. Finally, culture media was harvested and cleared of cellular debris by brief centrifugation. Fractional cholesterol efflux (expressed as a percentage) was calculated as the amount of radio-label detected in the supernatants divided by total radio-label in each well (radioactivity in the supernatant plus radioactivity in the cells) obtained after lipid extraction from cells in a mixture of 3:2 hexane:isopropanol (3:2 vol/vol). The background cholesterol efflux obtained in the absence of any acceptor was subtracted from the efflux obtained with samples. Flow cytometry Blood and spleen samples were collected at sacrifice for analysis of leukocyte subsets. Myeloid cells were identified as CD45+ CD11b+. Monocytes were identified as CD11b+ CD115+. Among them, classical monocytes were Gr1 high (or Ly6C high ) and non-classical monocytes were Gr1 low (or Ly6C low ). Neutrophils were identified as CD11b+ CD115-Gr1+ (or CD11b+ CD115-Ly6G+). B220 + IgM+ B lymphocytes, CD4+ and CD8+ T lymphocyte subsets were also analyzed. Antibodies raised against CD11b, CD115, Gr1 (Ly6C and G), B220, CD4, CD8a, NK1.1, CD45, F4/80, CD3ε, MHC II, IgM, CD11c, and CD36 were used for immunostaining and are listed in supplementary data 1 . Forward scatter (FSC) and side scatter (SSC) were used to gate live cells excluding red blood cells, debris, and cell aggregates in total blood cells and splenocytes preparations. Cells were acquired using a BD LSRII Fortessa flow cytometer (BD Biosciences) and analyzed with FlowJo™ (TreeStar, Inc.). Quantitative real-time PCR RNA extraction was done either with Trizol or with Qiagen columns (RNeasy MiniSpin Columns) using a polytron (T25 basic, IKA, Labortechnik). 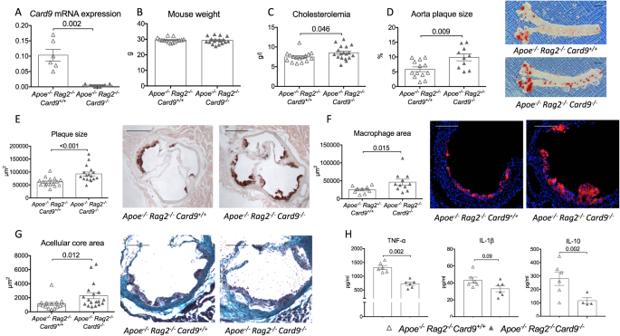Fig. 3: Card9 deficiency accelerates atherosclerosis in immunodeficientApoe-/-Rag2-/-mice. ACard9mRNA expression by peritoneal macrophages isolated from maleApoe-/-Rag2-/-Card9+/+andApoe-/-Rag2-/-Card9-/-mice (n= 6/group).BWeight at sacrifice after 6 weeks of fat diet (3 pooled experiments,n= 16–18/group).Cplasma cholesterol levels at sacrifice after 6 weeks of fat diet (3 pooled experiments,n= 14Apoe-/-Rag2-/-Card9+/+andn= 16Apoe-/-Rag2-/-Card9-/-).Drepresentative photomicrographs and quantitative analysis of atherosclerotic lesions on the thoraco-abdominal aorta of ofApoe-/-Rag2-/-Card9+/+andApoe-/-Rag2-/-Card9-/-mice after 6 weeks of fat diet (n= 6Apoe-/-Rag2-/-Card9+/+andn= 7Apoe-/-Rag2-/-Card9-/-);Erepresentative photomicrographs and quantitative analysis of atherosclerotic lesions in the aortic sinus ofApoe-/-Rag2-/-Card9+/+andApoe-/-Rag2-/-Card9-/-mice after 6 weeks of fat diet (3 experiments pooled,n= 14Apoe-/-Rag2-/-Card9+/+andn= 16Apoe-/-Rag2-/-Card9-/-); Scale bar 200 μm.Frepresentative photomicrographs and quantitative analysis of macrophage accumulation (MOMA staining, red) in atherosclerotic lesions ofApoe-/-Rag2-/-Card9+/+andApoe-/-Rag2-/-Card9-/-mice after 6 weeks of fat diet (3 experiments pooled,n= 14Apoe-/-Rag2-/-Card9+/+andn= 16Apoe-/-Rag2-/-Card9-/-); Scale bar 100 μm.GRepresentative photomicrographs and quantitative analysis of acellular area (Masson’s Trichrome) ofApoe-/-Rag2-/-Card9+/+andApoe-/-Rag2-/-Card9-/-mice after 6 weeks of fat diet (3 experiments pooled,n= 14Apoe-/-Rag2-/-Card9+/+andn= 16Apoe-/-Rag2-/-Card9-/-); Scale bar 100 μm.HCytokine production (ELISA) by Lps/Ifnγ-stimulated splenocytes isolated fromApoe-/-Rag2-/-Card9+/+andApoe-/-Rag2-/-Card9-/-mice (n= 6/group). Data are presented as mean values ±SD. Two-tailed Mann–Whitney test. Source data are provided as a Source Data file. The phase containing RNAs was then recuperated and washed with molecular biology water. RNA quality control and concentration were performed using Nanodrop 2000 (Thermofisher scientific). Reverse transcription was done following manufacturer instruction [kit QuantiTect Reverse Transcription (Qiagen)]. Real-time fluorescence monitoring was performed with the Applied Biosystems, Step One Plus Real-Time PCR System with Power SYBR Green PCR Master Mix (Eurogentec). qPCR was performed in triplicate for each sample. GAPDH cycle threshold was used to normalize gene expression: (F: 50 -CGTCCCGTAGACAAAATGGTGAA-30; R: 50 - GCC GTGAGTGGAGTCATACTGGAACA-30). Relative expression was calculated using the 2-delta-delta CT method followed by geometric average, as recommended. The following primer sequences were used: Card9 ( F: 5′- GAC CCT CTT AGT CCC AAT CTG -3′; R: 5′- CTC GTC GTC ATT CTC ATA GTC TG -3′), Mrs1 (F: 5′- CCG TGA ATC TAC AGC AAA GCA -3′; R: 5′- CCC AGT CCT TCA GTC TGA GG -3′), Scarb1 (F: 5′- CCT CCT GTT GCT GGT GCC CAT CAT -3′; R: 5′- GCA CTG GTG GGC TGT CCG CTG AGA -3′), Cd36 (F: 5′- TGG CCA AGC TAT TGC GAC ATG ATT A -3′; R: 5′- CGG GGA TTC CTT TAA GGT CGA TTT C -3′), Abcg1 (F: 5′- GAC AGC CAT CCC CGT CCT GCT CTT -3′; R: 5′- CTC CCG CAG GAT GGC CTC TGA CTT -3′), and Abca1 (F: 5′- GGC GGA CCT CCT GTG GTG TTT -3′; R: 5′- GAA TCT CCG GGC TTT AGG GTC CAT -3′). Transcriptomic analysis on human monocytes RNA sequencing libraries were prepared from 100 to 200 ng of total RNA using the Illumina® Stranded Total RNA Prep, Ligation with Ribo-Zero Plus library preparation kit, which allows performing a strand specific sequencing. This protocol includes a first step of enzymatic depletion of abundant transcripts from multiple species (including human cytoplasmic & mitochondria rRNA, mouse rRNA, rat rRNA, bacteria Gram +/- rRNA, human beta globin transcripts) using specific probes. cDNA synthesis was then performed and resulting fragments were used for dA-tailing followed by ligation of RNA Index Anchors. PCR amplification with indexed primers (IDT for Illumina RNA UD Indexes) was finally achieved, with 13 cycles, to generate the final cDNA libraries. Individual library quantification and quality assessment were performed using Qubit fluorometric assay (Invitrogen) with dsDNA HS (High Sensitivity) Assay Kit and LabChip GX Touch using a High Sensitivity DNA chip (Perkin Elmer). Libraries were then equimolarly pooled and quantified by qPCR using the KAPA library quantification kit (Roche). Sequencing was carried out on the NovaSeq 6000 instrument from Illumina using paired-end 2 × 100 bp, to obtain around 100 million clusters (200 million raw paired-end reads) per sample. Raw and normalized counts are provided in Supplementary data. We performed the gene set enrichment analysis using clusterProfiler v4.0.5 [54] with selected pathways from Gene Ontology (GO) and Kyoto Encyclopedia of Genes and Genomes (KEGG) databases, and Benjamini-Hochberg correction was applied. Used keywords were: “apopto*”, “atheroscleros*”, “NF-kappa B”, “TNF”. All pathways with adjusted p-value below 0.05 were considered as significantly enriched. For each category, median expression of all gene included in core enrichment were calculated for each patient before plotting the heatmap. Single-cell analysis of Card9/CARD9 expression patterns S ingle-cell RNA sequencing (scRNA-seq) datasets of immune cells from mouse aortic atherosclerotic plaques, reported in various publications [55] , [56] , [57] , [58] , [59] , [60] , [61] , (see ref. [34] for details), were pooled and integrated using canonical correlation analysis (CCA) in Seurat v4.3.0 [62] , [63] . All datasets used for analysis were pre-processed as follows: cells containing >200 detected genes, and genes detected in at least 3 cells were included in the analysis using the ‘CreateSeuratObject’ function with ‘min.features = 200’ and ‘min.cells=3’. Quality control filtering was further performed to remove dead/damaged cells with a high proportion of mitochondrial transcripts, and outlier cells with high UMI numbers (probable doublets/mutliplets). For mitochondrial transcripts, a < 5% cutoff was applied for all datasets, except for the data from Williams et al. [60] and from Gil-Pulido et al. [61] , where <7.5% and <10% cutoffs were applied, respectively. Pre-processing code for aortic leukocyte datasets can be found as supplemental files of Zernecke et al. [34] . All data were log normalized using the ‘NormalizeData’ function in Seurat with default parameters. Data integration was performed using a canonical CCA workflow in Seurat with default parameters. After CCA integration, data were scaled using ‘ScaleData’, and principal component analysis was performed using ‘RunPCA’. Dimensional reduction was performed using ‘RunUMAP’ with 30 principal components. Clustering was performed using ‘FindNeighbors’ with 30 principal components, and ‘FindClusters’ with a resolution of 0.4. Immune cell annotations are based on Zernecke’s works [34] , [64] . Mouse scRNA-seq data given in Supplementary Fig. 2 were obtained from Pan et al. [18] and downloaded from Gene Expression Omnibus GSE155513, pre-processed in cellranger-6.1.2, and further analyzed in Seurat v4.3.0 [63] . We used data from Ldlr -/- mice fed normal chow or a western diet for 8, 16 or 26 weeks (i.e. the following data from Gene Expression Omnibus GSE155513: GSM4705592, GSM4705593, GSM4705594, GSM4705595, GSM4705596, GSM4705597, GSM4705598, GSM4705599). Individual datasets were pre-processed with quality control filtering in Seurat: cells containing >200 detected genes, and genes detected in at least 3 cells were included in the analysis using the ‘CreateSeuratObject’ function with ‘min.features = 200’ and ‘min.cells = 3’. Quality control filtering was further performed to remove dead/damaged cells with a high proportion of mitochondrial transcripts (>10%), and outlier cells with high UMI numbers. All data were log normalized using the ‘NormalizeData’ function in Seurat with default parameters. Data were pooled and batch corrected using Harmony [65] within Seurat. 2000 highly variable genes were identified using ‘FindVariableFeatures’ (with selection.method = “vst”). Data were scaled using ‘ScaleData’ with default parameters, and principal component analysis performed using ‘RunPCA’ with default parameters, and batch corrected using ‘RunHarmony’ with default parameters. Dimensional reduction was performed using ‘RunUMAP(reduction = “harmony”, dims = 1:20)’, and clustering was performed at a 0.4 resolution using ‘FindNeighbors(reduction = “harmony”, dims = 1:20)’ followed by ‘FindClusters(resolution = 0.2)’. Positive marker genes for each cluster were identified using ‘FindAllMarkers’. Human scRNA-seq data given in Fig. 7 were obtained from total cells of human atherosclerotic coronary arteries [33] and analyzed in Seurat v3 [62] starting from the author provided cell-count matrix (downloaded from Gene Expression Omnibus GSE131778). Cells containing <200 detected genes were excluded, and genes detected in at least 3 cells were included in the analysis using the ‘CreateSeuratObject’ functions with ‘min.features = 200’ and ‘min.cells = 3’. Further quality control filtering was performed and cells with >5% mitochondrial transcripts were excluded, as well as cells with outlier number of UMIs (nCount_RNA > 15,000). A total of 10,934 cells were analyzed. As a pre-analysis indicated a substantial patient-driven batch effect, we performed batch correction using Harmony [65] within Seurat, considering each patient as an independent sample. Data were normalized using the ‘NormalizeData’ function in Seurat with default parameters. In all, 2000 highly variable genes were identified using ‘FindVariableFeatures’ (with selection.method = “vst”). Data were scaled using ‘ScaleData’ with default parameters, and principal component analysis performed using ‘RunPCA’ with default parameters, and batch corrected using ‘RunHarmony’ with default parameters. Dimensional reduction was performed using ‘RunUMAP(reduction = “harmony”, dims = 1:20)’, and clustering was performed at a 0.4 resolution using ‘FindNeighbors(reduction = “harmony”, dims = 1:20)’ followed by ‘FindClusters(resolution = 0.4)’. Positive marker genes for each cluster were identified using ‘FindAllMarkers’. Cell type annotation was performed based on expression of known cell lineage markers, and on cluster annotations in Wirka et al. 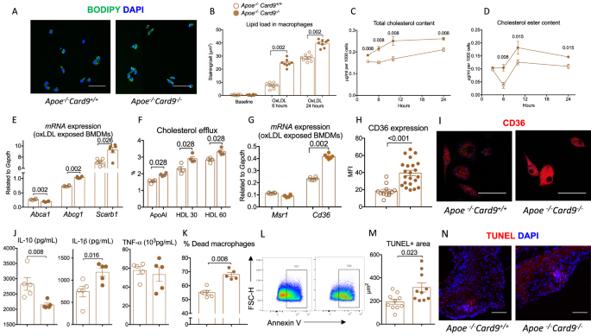Fig. 4:Card9deficiency increased CD36 expression in macrophages and promotes lipid uptake and foam cell formation. ARepresentative photomicrographs and quantitative analysis (B) of Bodipy+ foam cells after incubation of BMDMs fromApoe-/-Card9+/+andApoe-/-Card9-/-mice with oxLDL during 6 and 24 h (2 pooled experiments,n= 8/group/timepoints), Scale bar 10 μm.Cquantification of intracellular cholesterol content of BMDMs fromApoe-/-Card9+/+andApoe-/-Card9-/-mice after exposure to ox-LDL (n= 6/group/timepoint).DQuantification of intracellular cholesterol ester of BMDMs fromApoe-/-Card9+/+andApoe-/-Card9-/-mice after exposure to ox-LDL at 3, 6, 12, and 24 h (n= 6/group/timepoint).EQuantification ofAbca1andAbcg1andScarb1mRNA expression in BMDMs fromApoe-/-Card9+/+andApoe-/-Card9-/-mice after stimulation with oxLDL (n= 6/group).FQuantification of cholesterol efflux in presence of ApoAI or HDL (n= 4/group).GQuantification ofMrs1 and Cd36mRNAs in BMDMs fromApoe-/-Card9+/+andApoe-/-Card9-/-mice after stimulation with oxLDL (n= 6/group).H,Irepresentative immunostaining and quantification of Cd36 expression by BMDMs fromApoe-/-Card9+/+andApoe-/-Card9-/-mice after 24-h stimulation with ox-LDL (n= 12Apoe-/-Card9+/+andn= 22Apoe-/-Card9-/-), Scale bar 10 μm.Jcytokine production by BMDMs fromApoe-/-Card9+/+andApoe-/-Card9-/-mice after stimulation (ELISA in the supernatant,n= 5/group) and oxLDL exposure.K,LFlow cytometry quantification of AnnexinV+ BMDMs fromApoe-/-Card9+/+andApoe-/-Card9-/-mice after 24-h stimulation with oxLDL (100 μmol/l;n= 5/group).M,Nrepresentative photomicrographs and quantification of TUNEL+ cells in plaques fromApoe-/-Card9+/+andApoe-/-Card9-/-mice (n= 10/group). Scale bar 20 μm. Data are presented as mean values ±SD. Two-tailed Mann–Whitney test. Source data are provided as a Source Data file. [33] . In Supplementary Fig. 15e–g , the expression of CARD9 was examined in scRNA-seq data of mononuclear phagocytes from human coronary and carotid arteries in an integrated dataset described in details in Zernecke et al. [34] . Western blot Proteins from BMDMs were extracted by pipetting in ice-cold lysis buffer (NaCl 150 mM, HEPES 20 mM, EDTA 1 mM, EGTA 1 mM, NP-40 0.25% (Vol/Vol)) supplemented with protease (1 tab/10 ml, Roche) and phosphatase (Na 4 VO 3 2 mM) inhibitors). Protein extracts were briefly sonicated (5 pulses, amplitude 20, Vibracell 75021) and quantified by BCA (Thermofisher Scientific). Equal protein amounts were separated by SDS-PAGE (10% acrylamide) and transferred onto nitrocellulose membrane (0.2 μm, Biorad). For LC3b detection, SDS-PAGE separated proteins were transferred onto polyvinylidene difluoride membranes. Membranes were then blocked with Tris Buffered Saline supplemented with 0.1% Tween-20 (TBST) and 2% BSA (2 h at room temperature), then incubated with primary antibodies (overnight, 4 °C) diluted following the manufacturer’s recommendations. After three washes in TBST, membranes were incubated with species-specific horseradish peroxidase-conjugated secondary antibodies (1:8000 dilution, 45 min at room temperature). After three washes in TBST, the peroxidase activity was detected using Clarity Western ECL Substrate (Biorad) using Cytiva’s ImageQuant Fluor 800. The migration position of transferred proteins was compared to the PageRuler Prestain Protein Ladder (10 to 170 kDa, Thermo Fisher Scientific). Densitometric analysis was performed using ImageJ software (NIH). Phosphorylated protein signals were normalized on total protein levels, whereas non-phosphorylated proteins were normalized on β-actin protein levels. Primary and HRP-coupled secondary antibodies used for immunoblotting experiments are listed in supplementary data 3 . Uncropped Western blots are available as supplementary material. Microbiota analysis Stool collection and DNA extraction Fecal samples were homogenized and 0.2 g aliquots were stored at −80 °C for further analysis. DNA was extracted from fecal samples using a multi-step protocol [66] . Briefly, the feces samples were weighed and then resuspended for 10 min at room temperature in 250 μl of 4 M guanidine thiocyanate in 0.1 M Tris (pH 7.5) (Sigma-Aldrich) and 40 μl of 10% N-lauroyl sarcosine (Sigma-Aldrich). After the addition of 500 μl of 5% N-lauroyl sarcosine in 0.1 M phosphate buffer (pH 8.0), the 2-ml tubes were incubated at 70 °C for 1 h. One volume (750 ml) of a mixture of 0.1- and 0.6-mm-diameter silica beads (Sigma-Aldrich) (sterilized by autoclaving) was added, and the tube was shaken at 6.5 m/s three times for 30 s each in a FastPrep (MP Biomedicals) apparatus. Polyvinylpolypyrrolidone (15 mg) was added to the tube, which was then vortexed and centrifuged for 5 min at 20,000 × g . After recovery of the supernatant, the pellets were washed with 500 μl of TENP (50 mM Tris (pH 8), 20 mM EDTA (pH 8), 100 mM NaCl, 1% polyvinylpolypyrrolidone) and centrifuged for 5 min at 20,000 × g , and the new supernatant was added to the first supernatant. The washing step was repeated two times. The pooled supernatant (about 2 ml) was briefly centrifuged to remove particles and then split into two 2-ml tubes. Nucleic acids were precipitated by the addition of 1 volume of isopropanol for 10 min at room temperature and centrifugation for 10 min at 20,000× g . Pellets were resuspended and pooled in 450 μl of 100 mM phosphate buffer, pH 8, and 50 ml of 5 M potassium acetate. The tube was placed on ice overnight and centrifuged at 20,000 × g for 30 min. The supernatant was then transferred to a new tube containing 20 μl of RNase (1 mg/ml) and incubated at 37 °C for 30 min. Nucleic acids were precipitated by the addition of 50 μl of 3 M sodium acetate and 1 ml of absolute ethanol. The tube was incubated for 10 min at room temperature, and the nucleic acids were recovered by centrifugation at 20,000 × g for 15 min. The DNA pellet was finally washed with 70% ethanol, dried, and resuspended in 100 μl of Tris–EDTA (TE) buffer. Sequencing Microbiota analysis was performed by amplicon sequencing of the V3-V4 region of the 16 S ribosomal RNA gene. This region was amplified using the following primers – 16 S sense 5′-TACGGRAGGCAGCAG-3′ and anti-sense 5′-CTACCNGGGTATCTAAT-3′ – according to an optimized and standardized 16 S amplicon library preparation protocol (Metabiote, GenoScreen, Lille, France). Briefly, PCR of the 16 S DNA was performed with 5 ng of genomic DNA according to the manufacturer’s protocol (Metabiote), with bar-coded primers (Metabiote MiSeq Primers) to a final concentration of 0.2 μmol/l, with an annealing temperature of 50 °C for 30 cycles. Purification of the PCR products was performed with Agencourt AMPure XP-PCR purification system (Beckman Coulter, Brea, CA, USA), and quantified following the manufacturer’s instructions. The samples were multiplexed at equal concentrations. Sequencing was performed on an Illumina MiSeq platform (Illumina, San Diego, CA, USA) using a 250 bp paired-end sequencing protocol at GenoScreen. Raw paired-end reads were subjected to the following processes: (1) quality filtering using the PRINSEQ-lite PERL script [67] , by truncating the bases from the 3′ end, that did not exhibit a quality <30, based on the Phred algorithm and (2) searching for and removing both forward and reverse primer sequences using CutAdapt, with no mismatches allowed in the primer sequences. Only sequences where perfect matching forward and reverse primers were detected were included. 16S sequence analysis Sequences were quality filtered using the dada2 software package (version 1.12.1) [68] in the R programming language (R version 3.6.1) to produce amplicon sequence variants (ASVs). Taxonomic classification was performed using the Silva reference database (version 132) [69] . Bacterial ASVs that could not be assigned to Phylum-level taxonomy were excluded. 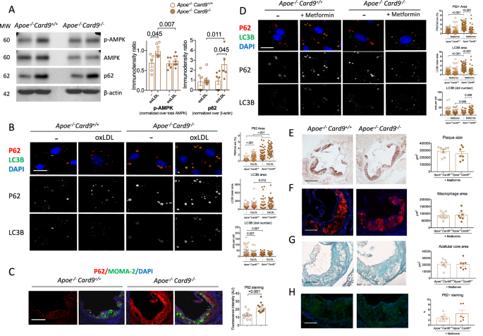Fig. 5: Pro-atherogenic effects ofCard9deficiency are mediated by impaired autophagy. AQuantitation of AMPK phosphorylation and p62 content in macrophages from fromApoe-/-Card9+/+(n= 5) andApoe-/-Card9-/-mice (n= 8) after exposure to oxLDL (western blot).Brepresentative photomicrographs and quantitative analysis and of p62 (Red), LC3B (Green) content in macrophages fromApoe-/-Card9+/+andApoe-/-Card9-/-mice at baseline and after exposure to oxLDL (n= 48 for p62 andn= 40 for LC3B).CQuantitative analysis and representative photomicrographs of p62 accumulation (Red) in MOMA-2+ macrophages (Green) in atherosclerotic lesions ofApoe-/-Card9+/+(n= 10) andApoe-/-Card9-/-mice (n= 12) after 6 weeks of fat diet (2 experiments pooled); Scale bar 200 μm.Drepresentative photomicrographs and quantitative analysis and of p62 (Red), LC3B (Green) content in ox-LDL exposed macrophages fromApoe-/-Card9+/+andApoe-/-Card9-/-mice treated or not with metformin (n= 48 for p62 andn= 40 for LC3B).E–Hcharacterization of atherosclerotic lesions in the aortic sinus of maleApoe-/-Card9+/+(n= 8)andApoe-/-Card9-/-mice (n= 7) after 6 weeks of fat diet and treated by metformin.Erepresentative photomicrographs and quantitative analysis of atherosclerotic lesions in the aortic sinus ofApoe-/-Card9+/+andApoe-/-Card9-/-mice after 6 weeks of fat diet and treated by metformin; Scale bar 200 μm.Frepresentative photomicrographs and quantitative analysis of macrophage accumulation (MOMA staining, red) in atherosclerotic lesions ofApoe-/-Card9+/+andApoe-/-Card9-/-mice after 6 weeks of fat diet and treated by metformin; Scale bar 100 μm.Grepresentative photomicrographs and quantitative analysis of acellular area (Masson’s Trichrome) ofApoe-/-Card9+/+andApoe-/-Card9-/-mice after 6 weeks of fat diet and treated by metformin; Scale bar 100 μm.Hrepresentative photomicrographs and quantitative analysis of p62 content (Green) in plaques ofApoe-/-Card9+/+andApoe-/-Card9-/-mice after 6 weeks of fat diet and treated by metformin; Scale bar 100 μm. Data are presented as mean values ±SD. Two-tailed Mann–Whitney test. Source data are provided as a Source Data file. Alpha diversity was estimated using the number of observed species and the Shannon diversity index. Raw sequence data are accessible in the Sequence Read Archive (accession number pending). Beta diversity analysis was performed on proportion-normalized data using the Bray-Curtis index. Assessment for significant differences between clusters was performed using PERMANOVA with the adonis function in the vegan package (version 2.5-6) in R with 99999 permutations. Differential abundance was tested using linear discriminant analysis with effect size (Lefse) using default settings [21] . LDL isolation and oxidation LDL from normal human pooled sera was prepared by ultracentrifugation and dialyzed against PBS containing 100 µM EDTA. 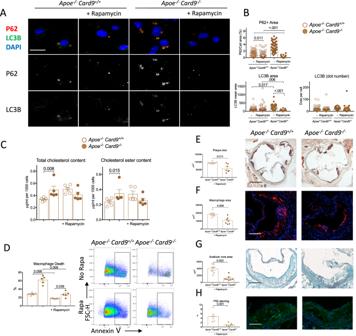Fig. 6: Protective effects of rapamycin in vitro and in vivo. A,Brepresentative photomicrographs and quantitative analysis of p62 (Red), LC3B (Green) content in oxLDL-exposed macrophages from maleApoe-/-Card9+/+andApoe-/-Card9-/-mice treated or not with rapamycin (200 mMol) (n= 48 for p62 andn= 40 for LC3B).Cquantification of intracellular cholesterol (total and ester) of BMDMs fromApoe-/-Card9+/+andApoe-/-Card9-/-mice after exposure to oxLDL with or without rapamycin (200 mMol) (n= 5/group).DFlow cytometry quantification of necrosis (7AAD+ Annexin V+) susceptibility of macrophages fromApoe-/-Card9+/+andApoe-/-Card9-/-mice after 24-h stimulation with high concentration of oxLDL (100 μmol/l) without and with rapamycin (200 mMol;n= 5/group).Erepresentative photomicrographs and quantitative analysis of atherosclerotic lesions in the aortic sinus ofApoe-/-Card9+/+andApoe-/-Card9-/-mice after 6 weeks of fat diet and treated by rapamycin (n= 7/group); Scale bar 200 μm.Frepresentative photomicrographs and quantitative analysis of macrophage accumulation (MOMA staining, red) in atherosclerotic lesions ofApoe-/-Card9+/+andApoe-/-Card9-/-mice after 6 weeks of fat diet and treated by rapamycin (n= 7/group; Scale bar 100 μm).Grepresentative photomicrographs and quantitative analysis of acellular area (Masson’s Trichrome) ofApoe-/-Card9+/+andApoe-/-Card9-/-mice after 6 weeks of fat diet and treated by rapamycin (n= 7/group; Scale bar 100 μm).Hrepresentative photomicrographs and quantitative analysis of p62 content (green) in plaques ofApoe-/-Card9+/+andApoe-/-Card9-/-mice after 6 weeks of fat diet and treated by rapamycin (n= 7/group; Scale bar 100 μm.). Data are presented as mean values ±SD. Two-tailed Mann–Whitney test. Source data are provided as a Source Data file. The LDL pool was then diluted to 2 g/l with PBS into a final volume of 3 ml. LDLs were mildly oxidized by UV-C for 2 h in the presence of 5 µM CuSO4 [70] . Oxidized LDL contained 4.2–7.4 nmoles of TBARS (thiobarbituric acid-reactive substances)/µg apoB. Relative electrophoretic mobility (REM) and 2,4,6-trinitrobenzenesulfonic acid (TNBS) reactive amino groups were 1.2–1.3 times and 85–92% of native LDL, respectively. Statistical analysis Graphs and statistical analyses were performed using Prism software (Graphpad). 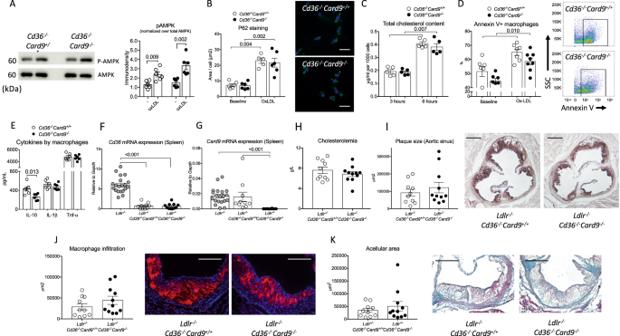Fig. 7: Pro-atherogenic effect of hematopoieticCard9deficiency was abolished in the absence of Cd36. Arepresentative blots and quantification of AMPK phosphorylation on BM-derived macrophages fromCd36-/-Card9+/+andCd36-/-Card9-/-macrophages after exposure to oxLDL (n= 6/group/condition).BQuantitative analysis and representative photomicrographs of P62 accumulation in macrophages fromCd36-/-Card9+/+andCd36-/-Card9-/-macrophages after 8-h exposure to oxLDL, Scale bar 100 μm (n= 6/group/condition).Cquantification of intracellular Cholesterol of BM-derived macrophages fromCd36-/-Card9+/+andCd36-/-Card9-/-mice after 3 and 6 h exposure to ox-LDL (n= 5/group/timepoint).DFlow cytometry quantification of Annexin V+ apoptotic BM-derived macrophages fromCd36-/-Card9+/+andCd36-/-Card9-/-mice after 24-h stimulation with high concentration of oxLDL (50 μmol/l; Baselinen= 6/group, OxLDLn= 7Cd36-/-Card9+/+andn= 8Cd36-/-Card9-/-).ECytokine production by BMDMs fromCd36-/-Card9+/+andCd36-/-Card9-/-mice after stimulation (ELISA in the supernatant,n= 6/group).FCd36mRNA expression in the spleen fromLdlr-/-mice and chimericLdlr-/-Cd36-/-Card9+/+andLdlr-/-Cd36-/-Card9-/-mice (n= 20/10/10).GCard9mRNA expression in the spleen fromLdlr-/-mice and chimericLdlr-/-Cd36-/-Card9+/+andLdlr-/-Cd36-/-Card9-/-mice (n= 20/10/10).H–Kcharacterization of chimeric maleLdlr-/-Cd36-/-Card9+/+(n= 10) andLdlr-/-Cd36-/-Card9-/-mice (n= 11).Hcholesterolemia in chimeric mice at sacrifice.Irepresentative photomicrographs and quantitative analysis of atherosclerotic lesions in the aortic sinus of chimericLdlr-/-Cd36-/-Card9+/+andLdlr-/-Cd36-/-Card9-/-mice after 8 weeks of fat diet; Scale bar 200 μm.Jrepresentative photomicrographs and quantitative analysis of macrophage accumulation (MOMA staining, red) in atherosclerotic lesions of chimericLdlr-/-Cd36-/-Card9+/+andLdlr-/-Cd36-/-Card9-/-mice after 8 weeks of fat diet; Scale bar 100 μm.KRepresentative photomicrographs and quantitative analysis of acellular area (Masson’s Trichrome) of chimericLdlr-/-Cd36-/-Card9+/+andLdlr-/-Cd36-/-Card9-/-mice after 8 weeks of fat diet; Scale bar 100 μm. Data are presented as mean values ±SD. Two-tailed Mann–Whitney test. Source data are provided as a Source Data file. 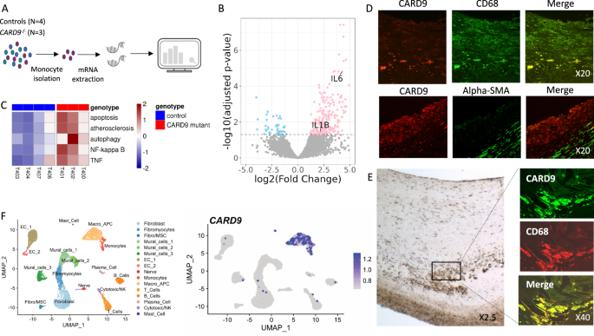Fig. 8: CARD9 related pathways in human. Aprotocol to obtain transcripts after isolation of monocytes from controls andCARD9-deficient patients.BVolcano-plot of the differentially expressed genes between monocytes from patients withCARD9mutation and control patients. Red dots represent up-regulated genes and blue dots down-regulated genes (adjustedp-value < 0.05).CHeatmap of mean expression in each patient of the leading edge genes contributing to the enrichment of indicated pathways in the GSEA. Immunofluorescent micrograph of human healthy (D) and atherosclerotic (E) carotid artery sections stained for CARD9 (green), α-actin + smooth muscle (red) or CD68 (red) showing that CARD9 was strongly expressed by cells that engulf lipids and cholesterol crystals and of giant lipid-laden foam cells but not by smooth muscle cells. Magnitude X20 (D), X2.5 (E), X40 (E) (2 Pooled experiments,n= 6/staining).FCARD9 expression in 10,934 total human atherosclerotic coronary artery cells from 4 patients (data from Wirka et al.33) with UMAP representation of single-cell RNA-seq gene expression data (left) and cellular lineage identification (right) where CARD9 expression in single cells projected onto the UMAP plot. (For clarity, expression cutoff have been applied and cells with detectable Card9/CARD9 transcripts were brought to the front of the plot). Values are expressed as mean ± s.e.m. Differences between values were examined using the nonparametric two-tailed Mann–Whitney, Kruskal–Wallis tests when appropriate and were considered significant at P < 0.05. Reporting summary Further information on research design is available in the Nature Portfolio Reporting Summary linked to this article.